Snf2h-mediated chromatin organization and histone H1 dynamics govern cerebellar morphogenesis and neural maturation Chromatin compaction mediates progenitor to post-mitotic cell transitions and modulates gene expression programs, yet the mechanisms are poorly defined. Snf2h and Snf2l are ATP-dependent chromatin remodelling proteins that assemble, reposition and space nucleosomes, and are robustly expressed in the brain. Here we show that mice conditionally inactivated for Snf2h in neural progenitors have reduced levels of histone H1 and H2A variants that compromise chromatin fluidity and transcriptional programs within the developing cerebellum. Disorganized chromatin limits Purkinje and granule neuron progenitor expansion, resulting in abnormal post-natal foliation, while deregulated transcriptional programs contribute to altered neural maturation, motor dysfunction and death. However, mice survive to young adulthood, in part from Snf2l compensation that restores Engrailed-1 expression. Similarly, Purkinje-specific Snf2h ablation affects chromatin ultrastructure and dendritic arborization, but alters cognitive skills rather than motor control. Our studies reveal that Snf2h controls chromatin organization and histone H1 dynamics for the establishment of gene expression programs underlying cerebellar morphogenesis and neural maturation. The importance of epigenetic regulation to brain development is recognized by the increasing number of developmental disorders caused by mutations in genes that encode proteins that modify or remodel chromatin structure [1] . Nonetheless, discerning precise mechanisms has proven challenging since these proteins impact all nuclear processes from transcription and replication to higher-order chromatin compaction. Genome-wide epigenetic profiling experiments have supported the hypothesis that neurogenesis is accompanied by the transition of a highly dynamic chromatin environment within progenitor cells to a more restrictive epigenetic landscape that dictates gene expression programs specific to each lineage [2] , [3] . Chromatin restriction involves the expansion of repressive histone marks such as H3K9Me3 and H3K27Me3, increased DNA methylation and a reduction in the distribution of the histone variant H2A.Z within gene bodies slated for silencing [4] , [5] . Concomitant with these histone and DNA modifications, chromatin compaction also requires regular nucleosome spacing and the inclusion of the linker histone H1 [6] , [7] . The repositioning of nucleosomes is catalysed by evolutionarily conserved multiprotein chromatin remodelling complexes (CRCs) that include a SNF2-domain containing catalytic subunit related to the Swi2/Snf2 family [8] . One such class of ATP-dependent nucleosome remodellers is the ISWI family, first identified in yeast [9] . Mammals have two ISWI homologues SNF2H ( SNF2 homologue ; human SMARCA5) and SNF2L ( SNF2-like ; human SMARCA1 ) that are the orthologs of yeast Isw1 and Isw2 genes [10] . ISWI can assemble regularly spaced nucleosomal arrays in vitro alone, or within a diverse number of protein complexes many of which contain a BAZ-family transcription factor (TF) [11] . ISWI complexes regulate many nuclear processes including DNA replication and repair (ACF, CHRAC and WICH), transcriptional regulation (NURF, RSF and CERF), and nucleolar structure and function (NoRC) [11] . ISWI inactivation in Drosophila also highlighted a role in higher-order chromatin structure [12] . However, despite a good understanding of the in vitro biochemical properties of ISWI and its related complexes, their in vivo roles remain poorly characterized. In the murine central nervous system (CNS), Snf2h and Snf2l display dynamic patterns of expression, where Snf2h expression peaks in neuronal progenitors, while Snf2l is expressed predominantly in terminally differentiated neurons [10] . For this reason, we postulated that Snf2h and Snf2l might regulate the transition from a progenitor to a differentiated neuron to restrict and compact chromatin while poising other genes for expression. In this regard, catalytically inactive Snf2l mice exhibit hypercellularity of cortical progenitors and delayed their differentiation, resulting in a larger brain [13] . However, Snf2h knockout (KO) mice die at the peri-implantation stage due to growth arrest of the trophoectoderm and inner cell mass, thereby preventing the study of Snf2h during brain development [14] . To overcome this problem we describe the generation of an Snf2h -targeted allele that facilitated its characterization throughout mouse brain development. Our studies reveal that Snf2h controls higher-order chromatin organization to mediate the establishment of gene expression programs underlying cerebellar morphogenesis and neural maturation. Snf2h and Snf2l are developmentally regulated in the cerebellum The closely related mammalian ISWI genes, Snf2h and Snf2l , display complementary expression patterns that suggest they have distinct roles during tissue development [10] . Embryonic brain mRNA and protein expression analyses reveals that Snf2h is robustly expressed in the developing rhombic lip, similarly to the hindbrain patterning TFs Engrailed-1 (En1) and Engrailed-2 (En2), whereas Snf2l expression was not detected within the rhombic lip at embryonic day (E) 14.5 ( Fig. 1a–e ). During late embryonic development, we observed robust Snf2h expression in developing Purkinje cells (PCs; Fig. 1f ), mature PCs ( Fig. 1g,i ) and in nearly all NeuroD1+ neural lineages ( Fig. 1h and Supplementary Fig. 1a,b ). In contrast, Snf2l expression was prominent only within PCs after P7 ( Fig. 1i and Supplementary Fig. 1c ). Immunoblots of hindbrain and cerebellar extracts demonstrated that Snf2h levels peaked during the period of granule neuron progenitor (GNP) proliferation (~E18 to P7), whereas Snf2l levels increased as a function of cerebellar maturity with peak expression after ~P10 ( Fig. 1j,k ). Interestingly, Snf2h downregulation after P7 coincides with En1 downregulation, whereas En2 expression is robust throughout cerebellar development ( Fig. 1j,k ). Expression of all proteins was maintained in adulthood, albeit at lower levels ( Fig. 1j,k ). We conclude that Snf2h is robustly expressed in hindbrain progenitors while Snf2h and Snf2l protein levels are dynamically modulated during post-natal development. 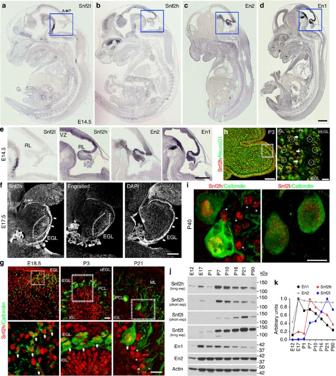Figure 1: Snf2h and Snf2l are dynamically regulated in the developing cerebellum. (a–d)In situhybridization for Snf2l, Snf2h, En2 and En1 from wild-type (WT) embryonic (E) 14.5 sagittal sections adapted from Genepaint.org70. Scale bar, 500 μm. (e) Boxed areas froma–dhighlight the robust expression of Snf2h, En2 and En1 within the developing rhombic lip, while Snf2l is not detectable. A, anterior; P, posterior. Scale bar, 200 μm. (f) E17.5 WT sagittal cerebellar sections serially immunolabelled with Snf2h and Pan-Engrailed (En) antibodies. Brackets highlight regions of robust Snf2h and Engrailed immunoreactivity (−ir). Arrows denote robust Snf2h-ir within the EGL. DAPI labels all nuclei. Scale bar, 200 μm. (g) Confocal Z-stacks through the WT cerebellar vermis co-labelled with Snf2h (red) and Calbindin (green), a marker of the PC lineage at the indicated ages. Boxed areas are enlarged at bottom. Arrows denote Snf2h+ PCs. Asterisks denote Snf2h+ interneurons at P21. EGL, external granule layer; IGL, internal granule layer; PCL, Purkinje cell layer; o, outer; i, inner. Scale bars, 20 μm (top panels); 10 μm (bottom panels). (h) Confocal Z-stacks through the WT cerebellar vermis at post-natal day 3 (P3) co-labelled with Snf2h (red) and NeuroD1 (green), a marker of differentiated neurons. Arrows denote NeuroD1+, Snf2h+ PCs, as distinguished by their nuclear size and laminar position. Circles denote NeuroD1+, Snf2h+ granule cells (GCs) within the iEGL and the IGL. Scale bar, 20 μm. (i) Confocal Z-stacks through the P40 WT cerebellar vermis co-labelled with calbindin (green) and Snf2h (red, left panel); or Snf2l (red, right panel). Asterisks denote Snf2h+ interneurons. Scale bar, 5 μm. At least three mice from each genotype were used for evaluation. (j) Snf2h, Snf2l, En1 and En2 immunoblots of WT cerebellar extracts, except for E12 and E17 where hindbrain extracts were used. Actin served as loading control. (k) Plot of relative Snf2h, Snf2l, En1 or En2 expression during cerebellar development. The peak expression for each protein was normalized to 1,n=3. Figure 1: Snf2h and Snf2l are dynamically regulated in the developing cerebellum. ( a – d ) In situ hybridization for Snf2l, Snf2h, En2 and En1 from wild-type (WT) embryonic (E) 14.5 sagittal sections adapted from Genepaint.org [70] . Scale bar, 500 μm. ( e ) Boxed areas from a – d highlight the robust expression of Snf2h, En2 and En1 within the developing rhombic lip, while Snf2l is not detectable. A, anterior; P, posterior. Scale bar, 200 μm. ( f ) E17.5 WT sagittal cerebellar sections serially immunolabelled with Snf2h and Pan-Engrailed (En) antibodies. Brackets highlight regions of robust Snf2h and Engrailed immunoreactivity (−ir). Arrows denote robust Snf2h-ir within the EGL. DAPI labels all nuclei. Scale bar, 200 μm. ( g ) Confocal Z-stacks through the WT cerebellar vermis co-labelled with Snf2h (red) and Calbindin (green), a marker of the PC lineage at the indicated ages. Boxed areas are enlarged at bottom. Arrows denote Snf2h+ PCs. Asterisks denote Snf2h+ interneurons at P21. EGL, external granule layer; IGL, internal granule layer; PCL, Purkinje cell layer; o, outer; i, inner. Scale bars, 20 μm (top panels); 10 μm (bottom panels). ( h ) Confocal Z-stacks through the WT cerebellar vermis at post-natal day 3 (P3) co-labelled with Snf2h (red) and NeuroD1 (green), a marker of differentiated neurons. Arrows denote NeuroD1+, Snf2h+ PCs, as distinguished by their nuclear size and laminar position. Circles denote NeuroD1+, Snf2h+ granule cells (GCs) within the iEGL and the IGL. Scale bar, 20 μm. ( i ) Confocal Z-stacks through the P40 WT cerebellar vermis co-labelled with calbindin (green) and Snf2h (red, left panel); or Snf2l (red, right panel). Asterisks denote Snf2h+ interneurons. Scale bar, 5 μm. At least three mice from each genotype were used for evaluation. ( j ) Snf2h, Snf2l, En1 and En2 immunoblots of WT cerebellar extracts, except for E12 and E17 where hindbrain extracts were used. Actin served as loading control. ( k ) Plot of relative Snf2h, Snf2l, En1 or En2 expression during cerebellar development. The peak expression for each protein was normalized to 1, n =3. Full size image Generation and characterization of Snf2h cKO mice To investigate the significance of ISWI expression changes within the cerebellum we proceeded to generate Snf2h conditional KO mice since Snf2h germline KO mice die at the peri-implantation stage [14] . We inserted loxP sites flanking exon 5, which encodes the evolutionarily conserved ATP-binding pocket critical for remodelling activity ( Fig. 2a,b ) [15] . Snf2h −/fl mice were bred with a Nestin-Cre driver line that demonstrated Cre expression in neural progenitors by ~E11 and displayed robust Cre activity in cerebellar progenitors during the early post-natal period ( Supplementary Fig. 2 ) [16] . Snf2h −/fl ::Nestin- Cre −/+ conditional KO mice ( Snf2h cKO-Nes hereon) were born at normal Mendelian ratios, but had a significant reduction in body weight by P7 ( Fig. 2c ), and were approximately half the size of control littermates by P20 ( Fig. 2d ). Brains isolated from these animals were reduced in size with striking cerebellar hypoplasia by P40 ( Fig. 2e ). Immunoblots of P0 cerebellar extracts confirmed an ~90% reduction in Snf2h protein levels ( Fig. 2f ). Three different behavioural assays demonstrated that Snf2h cKO mice have severe motor defects ( Fig. 2g ). We observed ataxia-like symptoms that began at ~P10, became severe by ~P15 to P20 and clearly contributed to the premature death of Snf2h cKO animals by ~P25 to P40 ( Fig. 2h and Supplementary Movies 1–5 ). Concomitantly, Snf2h −/fl mice bred onto our Snf2l −/Y line were then crossed with the Nestin-Cre driver line to generate animals deficient for both ISWI genes (Snf2h and Snf2l) [13] . However, these cDKO-Nes mice did not survive past birth ( Fig. 2h ). 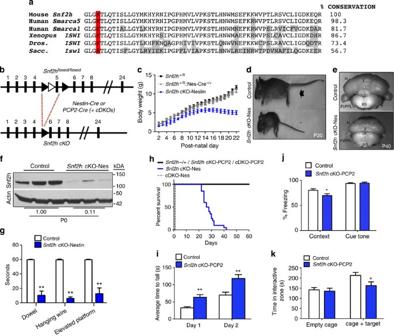Figure 2: Snf2h loss in cerebellar progenitors causes cerebellar ataxia or cognitive deficits when ablated in post-mitotic PCs. (a) Amino-acid conservation ofSnf2hexon 5 across species. The lysine residue within this ATP-binding motif and essential for catalytic activity is highlighted in red. Divergent amino acids are boxed grey.Xenopus,Xenopus laevis;Dros.,Drosophila melanogaster;Sacc.,Saccharomyces cerevisiae.(b) Schematic of the targeting strategy (LoxP sites, black arrowheads; Frt sites=white arrowheads) used to ablateSnf2hexpression using the Nestin-Cre or PCP2-Cre drivers. (c) Plot of body weights fromSnf2hcKO-Nes and control mice from P2 to P22. *P<0.05, one-way ANOVA,n=5–10. (d) Control (arrow) andSnf2hcKO-Nes (asterisk) littermates at P20. (e) Whole-mount images ofSnf2hcKO-Nes and control cerebella at P40. (f) Snf2h immunoblot fromSnf2hcKO-Nes and control cerebellar extracts at birth. Actin served as loading control. Values denote averaged densitometry,n=4. (g) Dowel, hanging wire and elevated platform tests reveal severe motor abnormalities inSnf2hcKO-Nes mice relative to control littermates at P20–P25. **P<0.01, one-way ANOVA,n=10–14. (h) Kaplan–Meier survival curves ofSnf2hcKO-Nes, cDKO-Nes and control littermates.Snf2hcKO-Nes mice were not viable under standard laboratory conditions after ~P30–P45, while cDKO-Nes mice did not survive past birth,n=20–30. (i) Rotarod test:Snf2hcKO-PCP2 exhibit enhanced ability to stay on the rotarod after five sessions of training relative to controls. **P<0.01, one-way ANOVA,n=10–14. (j) Fear conditioning test:Snf2hcKO-PCP2 exhibit no differences in freezing response during training, but a decreased freezing response in context-dependent learning relative to controls. *P<0.05, one-way ANOVA,n=10–14. (k) Social interaction test:Snf2hcKO-PCP2 exhibit reduced interaction time with a stranger mouse in a controlled social environment relative to control littermates. *P<0.05, one-way ANOVA,n=10–14. Values are presented as the mean±s.e.m. Figure 2: Snf2h loss in cerebellar progenitors causes cerebellar ataxia or cognitive deficits when ablated in post-mitotic PCs. ( a ) Amino-acid conservation of Snf2h exon 5 across species. The lysine residue within this ATP-binding motif and essential for catalytic activity is highlighted in red. Divergent amino acids are boxed grey. Xenopus , Xenopus laevis ; Dros ., Drosophila melanogaster ; Sacc ., Saccharomyces cerevisiae. ( b ) Schematic of the targeting strategy (LoxP sites, black arrowheads; Frt sites=white arrowheads) used to ablate Snf2h expression using the Nestin-Cre or PCP2-Cre drivers. ( c ) Plot of body weights from Snf2h cKO-Nes and control mice from P2 to P22. * P <0.05, one-way ANOVA, n =5–10. ( d ) Control (arrow) and Snf2h cKO-Nes (asterisk) littermates at P20. ( e ) Whole-mount images of Snf2h cKO-Nes and control cerebella at P40. ( f ) Snf2h immunoblot from Snf2h cKO-Nes and control cerebellar extracts at birth. Actin served as loading control. Values denote averaged densitometry, n =4. ( g ) Dowel, hanging wire and elevated platform tests reveal severe motor abnormalities in Snf2h cKO-Nes mice relative to control littermates at P20–P25. ** P <0.01, one-way ANOVA, n =10–14. ( h ) Kaplan–Meier survival curves of Snf2h cKO-Nes, cDKO-Nes and control littermates. Snf2h cKO-Nes mice were not viable under standard laboratory conditions after ~P30–P45, while cDKO-Nes mice did not survive past birth, n =20–30. ( i ) Rotarod test: Snf2h cKO-PCP2 exhibit enhanced ability to stay on the rotarod after five sessions of training relative to controls. ** P <0.01, one-way ANOVA, n =10–14. ( j ) Fear conditioning test: Snf2h cKO-PCP2 exhibit no differences in freezing response during training, but a decreased freezing response in context-dependent learning relative to controls. * P <0.05, one-way ANOVA, n =10–14. ( k ) Social interaction test: Snf2h cKO-PCP2 exhibit reduced interaction time with a stranger mouse in a controlled social environment relative to control littermates. * P <0.05, one-way ANOVA, n =10–14. Values are presented as the mean±s.e.m. Full size image To further elucidate the contribution of Snf2h to cerebellar function, we generated a second strain of Snf2h cKO mice using the PCP2-Cre driver line that becomes active specifically in post-mitotic PCs after P10 (ref. 17 ; Supplementary Fig. 3 ). Snf2h cKO-PCP2 and cDKO-PCP2 were both born at normal Mendelian ratios and survived into adulthood ( Fig. 2h ). As such, we assessed the performance of Snf2h cKO-PCP2 animals in a cohort of motor and cognitive behavioural assays. We observed an enhanced performance in the rotating rotarod ( Fig. 2i ), but no additional alterations in motor control or spatial learning ( Supplementary Fig. 4 ). In the fear-conditioning assay, the mice are exposed to a novel cue (cue tone), followed by a foot-shock (context), and the ‘fear’ response is measured (conditional response) [18] . Snf2h cKO-PCP2 mice had a normal response to the cue tone, but a reduced response to the context, suggestive of impaired associative learning skills ( Fig. 2j ). The social interaction assay measures the preference of mice to interact with a stranger mouse over an inanimate object. Snf2h cKO-PCP2 mice spent less time interacting with the stranger mouse than control littermates ( Fig. 2k ). We conclude that the loss of Snf2h in post-mitotic PCs does not result in motor deficits but rather in cognitive alterations. Snf2h loss affects GNP and PC progenitor expansion Since previous studies have highlighted a role for Snf2h-containing CRCs during DNA replication [19] , [20] , we assessed whether the cerebellar hypoplasia in Snf2h cKO-Nes mice resulted from poor GNP or PC expansion. First, we examined the expression of proliferation markers in GNPs residing in the external granule layer (EGL) at E17.5 and E18.5. This analysis revealed that the proportions of cycling (Ki67+), mitotic (phosphorylated histone H3+, pH3+) and S-phase (BrdU+) cells were specifically reduced in the EGL of Snf2h cKO-Nes embryos ( Fig. 3a–c ). The proliferation defects coincided with a dramatic increase in cell death, as shown by an increased number of TUNEL+ cells at E17 and P0 relative to controls ( Fig. 3c ). Moreover, measurements of the EGL showed that it was significantly reduced in size at P7 ( Fig. 3d ). Reduced proliferation in the Snf2h mutant cerebellum is in stark contrast to Snf2l deficient animals where we observed increased proliferation and delayed differentiation of cortical progenitors [13] . 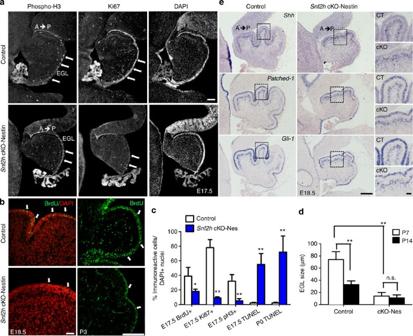Figure 3: Snf2h loss results in intrinsic GNP cell death without alteringShhsignalling. (a) E17.5 sagittal cerebellar sections fromSnf2hcKO-Nes and control littermates immunolabelled for phosphorylated Histone H3 (phospho-H3) or Ki67, and counterstained with the nuclear marker DAPI. Note a severe reduction of cells undergoing mitosis or S-phase throughout the mutant EGL (arrows). EGL, external granular layer. Scale bar, 100 μm. (b) Confocal Z-stacks through the E18.5 and P3 cerebellum fromSnf2hcKO-Nes and control littermates immunolabelled for BrdU after a 90-min BrdU-pulse (arrows). Scale bars, 100 μm. (c) Quantification of BrdU+, Ki67+, phospho-H3+ or TUNEL+ cells throughout the mutant and control EGL at E17.5 and P0. **P<0.01, Student’st-test,n=4. (d) EGL size at P7 and P14 inSnf2hcKO-Nes and control littermates. **P<0.01, student’st-test. n.s., not significant,n=4. Values are presented as the mean±s.e.m. for c,d. (e)In situhybridization through the cerebellar vermis from E18.5Snf2hcKO-Nes and control littermates forSonic Hedgehog(Shh), its receptorPatched-1, and their downstream targetGli-1.Note the spatiotemporal expression gradients (anterior high, posterior low) observed in both genotypes. Scale bar, 200 μm. Boxed areas are shown in rightmost panels to highlight robust mRNA levels in both genotypes. Scale bar, 50 μm. At least three mice from each genotype were used for evaluation. Figure 3: Snf2h loss results in intrinsic GNP cell death without altering Shh signalling. ( a ) E17.5 sagittal cerebellar sections from Snf2h cKO-Nes and control littermates immunolabelled for phosphorylated Histone H3 (phospho-H3) or Ki67, and counterstained with the nuclear marker DAPI. Note a severe reduction of cells undergoing mitosis or S-phase throughout the mutant EGL (arrows). EGL, external granular layer. Scale bar, 100 μm. ( b ) Confocal Z-stacks through the E18.5 and P3 cerebellum from Snf2h cKO-Nes and control littermates immunolabelled for BrdU after a 90-min BrdU-pulse (arrows). Scale bars, 100 μm. ( c ) Quantification of BrdU+, Ki67+, phospho-H3+ or TUNEL+ cells throughout the mutant and control EGL at E17.5 and P0. ** P <0.01, Student’s t -test, n =4. ( d ) EGL size at P7 and P14 in Snf2h cKO-Nes and control littermates. ** P <0.01, student’s t -test. n.s., not significant, n =4. Values are presented as the mean±s.e.m. for c,d. ( e ) In situ hybridization through the cerebellar vermis from E18.5 Snf2h cKO-Nes and control littermates for Sonic Hedgehog ( Shh ), its receptor Patched-1 , and their downstream target Gli-1. Note the spatiotemporal expression gradients (anterior high, posterior low) observed in both genotypes. Scale bar, 200 μm. Boxed areas are shown in rightmost panels to highlight robust mRNA levels in both genotypes. Scale bar, 50 μm. At least three mice from each genotype were used for evaluation. Full size image It is well established that the signalling factor Sonic Hedgehog ( Shh ) is secreted from PCs and plays a key role during GNP expansion and cerebellar foliation [21] , [22] , [23] . To assess whether poor GNP proliferation resulted from impaired Shh signalling, we examined the expression of Shh and its receptor, Patched-1 , as well as the downstream effectors Gli-1 , CyclinD1 and N-Myc by in situ hybridization. Sagittal sections through the cerebellar vermis from E18.5 Snf2h cKO-Nes and control littermates showed that surviving PCs secrete Shh normally, and that all downstream targets are activated in surviving GNPs ( Fig. 3e and Supplementary Fig. 5a ). To investigate PC progenitor proliferation, we birthdated cells by BrdU injection at E12.5 and harvested embryos at E17.5 for analysis [24] . Snf2h cKO-Nes embryos showed a significant reduction in the proportion of BrdU+, Calbindin+ PCs relative to controls ( Fig. 4a,d ). Additionally, BrdU-birthdating at E18.5 with analysis at P7 revealed that reduced GNP proliferation in Snf2h cKO-Nes mice resulted in a dramatic reduction in the number of BrdU+ GCs but not Calbindin+ PCs, residing within the internal granule layer (IGL), relative to controls ( Fig. 4b ). However, co-staining with Pax6 and NeuN demonstrated that the timing of neuronal differentiation was not affected ( Fig. 4c ). Moreover, a normal percentage of BrdU+, GFAP+ glial cells within the white matter suggested that the reduced cellular output was specific to neurons ( Fig. 4d and Supplementary Fig. 5b ). 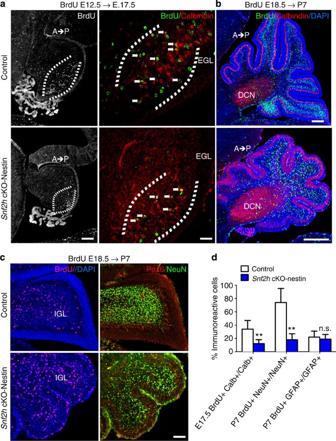Figure 4: Snf2h loss affects PC and GNP expansion resulting in cerebellar hypoplasia. (a) Confocal Z-stacks fromSnf2hcKO-Nes and control littermates that were BrdU-birthdated at E12.5, a time of PC birth, and co-labelled for BrdU (green) and Calbindin (red) at E17.5 (brackets). Note the reduction of BrdU+, Clabindin+PCs in mutant embryos (arrows). Scale bar, 50 μm. (b) Confocal Z-stacks fromSnf2hcKO-Nes and control littermates that were BrdU-birthdated at E18.5, a time of robust GNP expansion, and co-labelled for BrdU (green) and Calbindin (red) at P7. DAPI (blue) stains all nuclei. Note the spatiotemporal (anterior low, posterior high) distribution of BrdU+ GCs throughout the internal granule layer in control cerebella that is altered in mutant brains. DCN, deep cerebellar nuclei. Scale bar, 100 μm. (c) Confocal Z-stacks through the cerebellar vermis fromSnf2hcKO-Nes and control littermates that were BrdU-birthdated at E18.5, and labelled for BrdU (magenta); or co-labelled for Pax6 (red) and NeuN (green) at P7. DAPI (blue) stains all nuclei. Scale bar, 50 μm. At least three mice from each genotype were used for evaluation. (d) Quantification of double-labelled BrdU+ and Calbindin+ PCs at E17.5 (E12.5 BrdU birthdating); double-labelled BrdU+ and NeuN+ GCs at P7 (E18.5 BrdU-birthdating); or double-labelled BrdU+ and GFAP+ glial cells from mutant and control mice at P7 (E18.5 BrdU-birthdating). **P<0.01, Student’st-test. n.s., not significant,n=3. Values are presented as the mean±s.e.m. Figure 4: Snf2h loss affects PC and GNP expansion resulting in cerebellar hypoplasia. ( a ) Confocal Z-stacks from Snf2h cKO-Nes and control littermates that were BrdU-birthdated at E12.5, a time of PC birth, and co-labelled for BrdU (green) and Calbindin (red) at E17.5 (brackets). Note the reduction of BrdU+, Clabindin+PCs in mutant embryos (arrows). Scale bar, 50 μm. ( b ) Confocal Z-stacks from Snf2h cKO-Nes and control littermates that were BrdU-birthdated at E18.5, a time of robust GNP expansion, and co-labelled for BrdU (green) and Calbindin (red) at P7. DAPI (blue) stains all nuclei. Note the spatiotemporal (anterior low, posterior high) distribution of BrdU+ GCs throughout the internal granule layer in control cerebella that is altered in mutant brains. DCN, deep cerebellar nuclei. Scale bar, 100 μm. ( c ) Confocal Z-stacks through the cerebellar vermis from Snf2h cKO-Nes and control littermates that were BrdU-birthdated at E18.5, and labelled for BrdU (magenta); or co-labelled for Pax6 (red) and NeuN (green) at P7. DAPI (blue) stains all nuclei. Scale bar, 50 μm. At least three mice from each genotype were used for evaluation. ( d ) Quantification of double-labelled BrdU+ and Calbindin+ PCs at E17.5 (E12.5 BrdU birthdating); double-labelled BrdU+ and NeuN+ GCs at P7 (E18.5 BrdU-birthdating); or double-labelled BrdU+ and GFAP+ glial cells from mutant and control mice at P7 (E18.5 BrdU-birthdating). ** P <0.01, Student’s t -test. n.s., not significant, n =3. Values are presented as the mean±s.e.m. Full size image Taken together, these results suggest that the extrinsic cues (that is, Shh pathway) for progenitor expansion are unaltered and that the poor GNP and PC expansion in Snf2h cKO-Nes mice results from a cell-intrinsic defect, most likely from known ISWI functions in transcriptional regulation and DNA replication. Snf2h and Snf2l co-modulate the En1 locus In Drosophila , ISWI binding is enriched at transcriptional start sites where it influences gene transcription by repositioning nucleosomes [25] . We reasoned that altered nucleosome spacing within key developmental genes might perturb their expression and contribute to the impaired cerebellar development in the Snf2h cKO-Nes mice. Array hybridization of RNA isolated from mutant and control cerebella identified 110 genes differentially expressed at P0 that increased to 2,916 transcripts at P10 ( P <0.01, n =3 per genotype, statistics was carried out using WEBARRAY online tool ( http://www.webarraydb.org/webarray/index.html ), which utilizes linear model statistical analysis (modified t -test)). Gene ontology analysis using the DAVID online tool ( http://david.abcc.ncifcrf.gov/ ) revealed significant enrichment ( P <0.05) for downregulated genes associated with transcriptional regulation, cell adhesion and pattern specification ( Fig. 5 ). We further filtered our P0 and P10 microarrays with publicly available RNA-Seq data from isolated adult PCs, GCs and Bergmann glia, to assign a specific cerebellar cell type to the gene expression changes observed, where possible (for example, GNP/GC expression: En2 , Pax6, Uncx and NeuroD1 ; PC expression: protocadherin-ß (Pcdh-ß) isoforms; Supplementary Data 1 ) [26] . Validation of the microarray results by qRT–PCR confirmed that the expression of the TFs Rfx3 , Uncx , Cbp , Math1 , Pax6 , En2 , En1 ; the signalling factor Bmp4 and the cell adhesion molecules Pcdh-ß6 and Pcdh-ß17 were all significantly downregulated (~1.5–2.5-fold) in mutant cerebella at birth ( Fig. 6a ; Supplementary Table 1 ). Moreover, we observed a ~2.6-fold downregulation of Snf2h , while Snf2l levels were unperturbed in mutant cerebella at this time point ( Fig. 6a ). While most genes analysed remained downregulated at P10, we observed an unexpected increase in En1 (~1.9-fold), Bmp4 (~2.1-fold) and Snf2l (~1.7-fold) mRNA levels ( Fig. 6a ), the latter suggesting that Snf2l may be compensating for Snf2h loss in the activation of some targets. In this regard, P10 immunoblots demonstrated that Snf2l protein levels were increased by ~2.3-fold, whereas Snf2h protein levels were decreased by ~2-fold ( Fig. 6b ). Snf2l immunolabelling at P7 revealed comparable expression levels throughout the PC layer ( Fig. 6c ). We next investigated whether Snf2l could be responsible for the upregulation of genes at P10 that were reduced at P0, focusing our attention on En1. 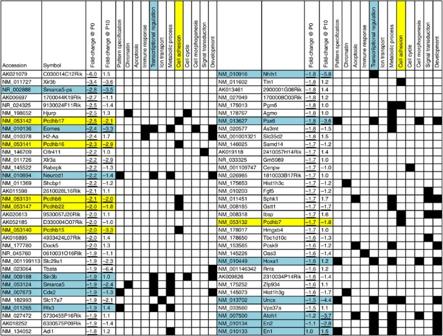Figure 5: List of downregulated genes at P0 and corresponding gene expression changes at P10 fromSnf2hcKO-Nes cerebella. Cyan highlights TFs and yellow highlights cell adhesion molecules. Note that ~110 genes were deregulated at P0, while ~2,900 genes were deregulated by P10. Three microarrays per genotype were averaged from wild-type and mutant P0 and P10 cerebellar extracts. Underlined values denoteP<0.05. Statistics was carried out using WEBARRAY online tool (http://www.webarraydb.org/webarray/index.html) that utilizes linear model statistical analysis (modifiedt-test). Figure 5: List of downregulated genes at P0 and corresponding gene expression changes at P10 from Snf2h cKO-Nes cerebella. Cyan highlights TFs and yellow highlights cell adhesion molecules. Note that ~110 genes were deregulated at P0, while ~2,900 genes were deregulated by P10. Three microarrays per genotype were averaged from wild-type and mutant P0 and P10 cerebellar extracts. Underlined values denote P <0.05. Statistics was carried out using WEBARRAY online tool ( http://www.webarraydb.org/webarray/index.html ) that utilizes linear model statistical analysis (modified t -test). 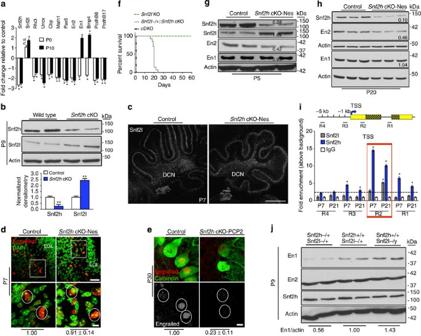Figure 6: Snf2h and Snf2l co-modulate theEn1locus. (a) RT–qPCR analysis of selected genes fromSnf2hcKO-Nes and control cerebella at P0 and P10. *P<0.05, Student’st-test. n.s., not significant,n=6 from one of two independent experiments. (b) Immunoblots for Snf2h and Snf2l fromSnf2hcKO-Nes and control cerebellar extracts at P9. Graph below depicts quantification for Snf2h and Snf2l, normalized to actin. **P<0.01, Student’st-test,n=3. Values are presented as the mean±s.e.m. (c,d) Confocal Z-stacks of P7 cerebellum fromSnf2hcKO-Nes and controls immunolabelled for (c) Snf2l. DCN, deep cerebellar nuclei. Scale bar, 200 μm; or (d) Pan-Engrailed (red) and counterstained with DAPI (green). Boxed areas are enlarged at bottom and denote similar En immunoreactivity in cells from both genotypes. Scale bars, 50 μm (top); 10 μm (bottom). (e) Confocal Z-stacks of P30 cerebellum fromSnf2hcKO-PCP2 and controls immunolabelled with Pan-Engrailed (red) and Calbindin (green). Engrailed images in bottom panel are pseudocolored (silver) for contrast. Scale bar, 5 μm. Values (d,e) denote Engrailed immunopixels normalized to WT within cells with a nuclear size >10 μm2(circles). At least 50 PCs from three independent mice were quantified per genotype. (f) Kaplan–Meier curves ofSnf2lKO,Snf2l−/+::Snf2hcKO-Nes and cDKO-Nes mice. Note that oneSnf2lallele in aSnf2h-null background rescues the lethality of cDKO-Nes mice up to ~P25 (n=25). (g,h) Immunoblots for Snf2l, Snf2h, En2 and En1 fromSnf2hcKO-Nes and control cerebellar extracts at P5 (g) and P20 (h). Actin served as loading control. Values denote averaged densitometry (n=4). (i) Top: schematic diagram of the mouseEn1locus indicating primer set locations. Yellow boxes, 5′ and 3′ untranslated regions (UTRs); striped yellow boxes, coding region; black line=non-coding region; TSS, transcription start site (arrow); kb, kilobases away from the TSS (+1). Bottom: ChIP-qPCR from WT cerebellar extracts for theEn1locus reveals Snf2h enrichment throughout the gene (R3, R2 and R1) at P7 and P21. Snf2l enrichment occurs only in the 5′-UTR (R2) at P21. *P<0.05, Student’st-test,n=4 from one of three independent experiments. Values are presented as the mean±s.e.m. (j) Immunoblots for Snf2h, En2 and En1 fromSnf2h+/+::Snf2l−/+(WT);Snf2h−/+::Snf2l−/+(Snf2h heterozygote); orSnf2h+/+::Snf2l−/y(Snf2l KO) cerebellar extracts at P9. Values denote averaged densitometry relative to WT levels (n=4). Full size image Figure 6: Snf2h and Snf2l co-modulate the En1 locus. ( a ) RT–qPCR analysis of selected genes from Snf2h cKO-Nes and control cerebella at P0 and P10. * P <0.05, Student’s t -test. n.s., not significant, n =6 from one of two independent experiments. ( b ) Immunoblots for Snf2h and Snf2l from Snf2h cKO-Nes and control cerebellar extracts at P9. Graph below depicts quantification for Snf2h and Snf2l, normalized to actin. ** P <0.01, Student’s t -test, n =3. Values are presented as the mean±s.e.m. ( c , d ) Confocal Z-stacks of P7 cerebellum from Snf2h cKO-Nes and controls immunolabelled for ( c ) Snf2l. DCN, deep cerebellar nuclei. Scale bar, 200 μm; or ( d ) Pan-Engrailed (red) and counterstained with DAPI (green). Boxed areas are enlarged at bottom and denote similar En immunoreactivity in cells from both genotypes. Scale bars, 50 μm (top); 10 μm (bottom). ( e ) Confocal Z-stacks of P30 cerebellum from Snf2h cKO-PCP2 and controls immunolabelled with Pan-Engrailed (red) and Calbindin (green). Engrailed images in bottom panel are pseudocolored (silver) for contrast. Scale bar, 5 μm. Values ( d , e ) denote Engrailed immunopixels normalized to WT within cells with a nuclear size >10 μm 2 (circles). At least 50 PCs from three independent mice were quantified per genotype. ( f ) Kaplan–Meier curves of Snf2l KO, Snf2l−/+::Snf2h cKO-Nes and cDKO-Nes mice. Note that one Snf2l allele in a Snf2h -null background rescues the lethality of cDKO-Nes mice up to ~P25 ( n =25). ( g , h ) Immunoblots for Snf2l, Snf2h, En2 and En1 from Snf2h cKO-Nes and control cerebellar extracts at P5 ( g ) and P20 ( h ). Actin served as loading control. Values denote averaged densitometry ( n =4). ( i ) Top: schematic diagram of the mouse En1 locus indicating primer set locations. Yellow boxes, 5′ and 3′ untranslated regions (UTRs); striped yellow boxes, coding region; black line=non-coding region; TSS, transcription start site (arrow); kb, kilobases away from the TSS (+1). Bottom: ChIP-qPCR from WT cerebellar extracts for the En1 locus reveals Snf2h enrichment throughout the gene (R3, R2 and R1) at P7 and P21. Snf2l enrichment occurs only in the 5′-UTR (R2) at P21. * P <0.05, Student’s t -test, n =4 from one of three independent experiments. Values are presented as the mean±s.e.m. ( j ) Immunoblots for Snf2h, En2 and En1 from Snf2h +/+ ::Snf2l −/+ (WT); Snf2h −/+ ::Snf2l −/+ (Snf2h heterozygote); or Snf2h +/+ ::Snf2l −/y (Snf2l KO) cerebellar extracts at P9. Values denote averaged densitometry relative to WT levels ( n =4). Full size image The En1 and En2 homeobox genes are essential for cerebellar patterning and foliation [27] . During early post-natal development they adopt distinct expression patterns with En1 and En2 expressed in PCs and GCs, respectively [28] . Since Snf2l expression is limited to PCs ( Fig. 1i and Supplementary Fig. 1c ), we reasoned that upregulation of En1 but not En2 might occur from Snf2l compensation. P7 sections through the cerebellar vermis were labelled with pan-Engrailed (Engrailed) antibodies, counterstained with DAPI and quantified for Engrailed immunoreactivity (-ir) within PCs (identified by their large nuclear size, >10 μm) from a minimum of 50 cells per genotype. We found that Snf2h cKO-Nes and control PC nuclei showed no significant differences in Engrailed-ir ( Fig. 6d ). However, the PCs of Snf2h cKO-PCP2 mice showed a significant reduction in Engrailed-ir, suggesting that Snf2l compensation is temporally regulated ( Fig. 6e ). Given that Snf2l compensates for embryonic Snf2h loss, we next investigated whether reducing Snf2l levels would increase the severity of the phenotype. Indeed, removal of one copy of Snf2l on the Snf2h cKO-Nes background ( Snf2l −/+ ::Snf2h cKO-Nes) resulted in a more severe ataxic phenotype and death by ~P25 ( Fig. 6f and Supplementary Movie 6 ). As discussed earlier, the cDKO-Nes mice had the most severe phenotype, resulting in death at birth ( Fig. 6f ), which is comparable to the neonatal lethality of En1 KO mice [29] . Microarray and immunostaining suggested that the Snf2l compensation begins between P0 and P7. Using immunoblots we were able to demonstrate En1 compensation as early as P5 with En2 expression reduced by ~60% ( Fig. 6g ). Similar results were observed at P20, suggesting that both ISWI proteins mediate En1 regulation, but En2 regulation is specific to Snf2h ( Fig. 6h ). Furthermore, P5 immunoblots show reduced En1 levels in the Snf2l −/+ ::Snf2h cKO-Nes animals compared with Snf2h cKO-Nes mice, thus providing additional support for a Snf2l -dependent En1 compensation in Snf2h cKO-Nes mice ( Supplementary Fig. 6a ). To determine the interactions at the En1 gene in vivo , we performed chromatin immunoprecipitation (ChIP) followed by quantitative PCR (ChIP–qPCR) assays for Snf2h and Snf2l with wild-type cerebellar extracts at P7, when Snf2h levels are at their peak; and at P21, when Snf2l levels reach their maximal level. En1 occupancy was analysed by qPCR with primer pairs corresponding to the intragenic region (R1), the 5′-UTR (R2), the proximal promoter (R3) and an upstream region (R4) ( Fig. 6i ). Snf2h binding showed the greatest enrichment at R2 at both time points with maximal binding observed at P7 ( Fig. 6i ). At P21, we also observed significant binding of Snf2l at R2 ( Fig. 6i ), suggesting that the ISWI proteins co-regulate En1 transcription and that increased Snf2l expression provides functional compensation in Snf2h cKO-Nes mice. In contrast, only Snf2h was enriched at the En2 promoter ( Supplementary Fig. 6b ), providing further support for Snf2h -specific regulation of En2 . As a last step to understand the endogenous function of Snf2h and Snf2l during normal cerebellar development, we assessed En1 and En2 expression levels upon deletion of one Snf2h allele ( Snf2h +/+ versus Snf2h −/+ ) or upon complete ablation of Snf2l ( Snf2l −/y versus Snf2l −/+ ) . Snf2h −/+ cerebella had a ~40% reduction of En1 total protein levels, while En2 and Snf2h protein levels were unaffected ( Fig. 6j ). Conversely, Snf2l deletion ( Snf2l −/y ; Snf2l is X-linked) resulted in a ~40% upregulation of En1 protein levels, while En2 and Snf2h protein levels remained unchanged ( Fig. 6j ). Collectively, our results suggest that when both Snf2h and Snf2l are present the endogenous role of Snf2l is to function as a repressor of En1 transcription, as En1 protein levels are increased in Snf2l KO cerebella at P9. However, when Snf2h is ablated embryonically ( Snf2h cKO-Nes model) we observed an upregulation of Snf2l that functionally compensates to restore En1 expression and early PC functions (probably by substitution within Snf2h complexes). However, this novel gain-of-function effect by Snf2l is temporally regulated since it does not rescue En1 expression when Snf2h is ablated at P10 (Snf2h cKO-PCP2 model). Moreover, Snf2l restoration of En1 expression within the Snf2h cKO-Nes mice is insufficient to rescue the progressive ataxic phenotype. Snf2h loss alters PC maturation The post-natal survival and progressive phenotype of Snf2h cKO-Nes mice allowed us to investigate the cell-intrinsic defects present in surviving post-mitotic neurons. For this analysis we chose the P7 cerebellum, a time when PC dendritic arbors extend towards the molecular layer for formation of parallel fibre circuits, while GCs migrate to the internal granule layer for establishment of mossy fibre circuitry [24] . We validated the loss of Snf2h in nearly all surviving Calbindin+ PCs ( Fig. 7a ), which were present in multiple PC layers compared with control PCs that were present in uniform developing rows ( Fig. 7b ). The growth of the molecular layer, which rapidly occurs between P7 and P14, was significantly reduced in size in the mutant animals ( Fig. 7d ). Indeed, a dramatic reduction of the PC apical dendritic arbor is observed with Golgi–Cox staining at P20, which is further aggravated in cDKO-Nes mice ( Fig. 7c,f ). In addition, we also observed a progressive and dose-dependent increase in the total number of PC pyknotic nuclei as assessed by toluidine blue staining ( Fig. 7e ). 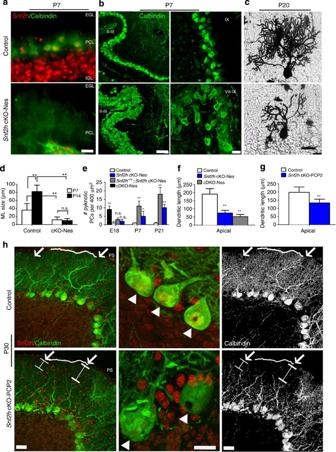Figure 7: Snf2h loss alters PC maturation. (a) Snf2h (red) and Calbindin (green) co-labelling through the cerebellum fromSnf2hcKO-Nes and control littermates at P7. Note the absence of Snf2h expression in mutant PCs. Scale bar, 20 μm. (b) Confocal Z-stacks through the cerebellar vermis fromSnf2hcKO-Nes and control littermates at P7 immunolabelled for Calbindin (green). Roman numerals denote the corresponding lobules of the mammalian cerebellum. Scale bars, 100 μm (left panels); 20 μm (right panels). (c) Light microscopy Z-stacks of PCs through the cerebellar vermis stained with the Golgi–Cox method fromSnf2hcKO-Nes mice and control littermates at P20. Scale bar, 10 μm. (d) Molecular layer size at P7 and P14 inSnf2hcKO-Nes and control littermates. (e) Quantification of pyknotic PC nuclei using toluidine blue reveals an ISWI-dependent modulation of PC survival inSnf2hcKO-Nes,Snf2l−/+::Snf2hcKO-Nes and cDKO-Nes mice. (f,g) PC apical arbor dendritic length measurements from the indicated genotypes at P20 or P30, respectively. For panels (d–g) **P<0.01, Student’st-test, n.s., not significant,n=6. Values are presented as the mean±s.e.m. (h) Left panels: confocal Z-stacks through the cerebellum from P30Snf2hcKO-PCP2 mice and control littermates co-immunolabelled for Snf2h (red) and calbindin (green). Arrows and bars denote mutant PC arbors that do not reach the pial surface (ps) (bars, arrows). Middle panels: higher magnification images of PCs (arrowheads) denote Snf2h+ staining in control but not mutant PCs. Right panels: pseudocolored Calbindin-ir (silver) denotes the atrophied dendritic arbor in mutant PCs (bars, arrows). Scale bar, 20 μm (left and rightmost panels); 10 μm (middle panels). Fora–candh, at least three mice from each genotype were used for evaluation. Figure 7: Snf2h loss alters PC maturation. ( a ) Snf2h (red) and Calbindin (green) co-labelling through the cerebellum from Snf2h cKO-Nes and control littermates at P7. Note the absence of Snf2h expression in mutant PCs. Scale bar, 20 μm. ( b ) Confocal Z-stacks through the cerebellar vermis from Snf2h cKO-Nes and control littermates at P7 immunolabelled for Calbindin (green). Roman numerals denote the corresponding lobules of the mammalian cerebellum. Scale bars, 100 μm (left panels); 20 μm (right panels). ( c ) Light microscopy Z-stacks of PCs through the cerebellar vermis stained with the Golgi–Cox method from Snf2h cKO-Nes mice and control littermates at P20. Scale bar, 10 μm. ( d ) Molecular layer size at P7 and P14 in Snf2h cKO-Nes and control littermates. ( e ) Quantification of pyknotic PC nuclei using toluidine blue reveals an ISWI-dependent modulation of PC survival in Snf2h cKO-Nes, Snf2l −/+ ::Snf2h cKO-Nes and cDKO-Nes mice. ( f,g ) PC apical arbor dendritic length measurements from the indicated genotypes at P20 or P30, respectively. For panels ( d – g ) ** P <0.01, Student’s t -test, n.s., not significant, n =6. Values are presented as the mean±s.e.m. ( h ) Left panels: confocal Z-stacks through the cerebellum from P30 Snf2h cKO-PCP2 mice and control littermates co-immunolabelled for Snf2h (red) and calbindin (green). Arrows and bars denote mutant PC arbors that do not reach the pial surface (ps) (bars, arrows). Middle panels: higher magnification images of PCs (arrowheads) denote Snf2h+ staining in control but not mutant PCs. Right panels: pseudocolored Calbindin-ir (silver) denotes the atrophied dendritic arbor in mutant PCs (bars, arrows). Scale bar, 20 μm (left and rightmost panels); 10 μm (middle panels). For a – c and h , at least three mice from each genotype were used for evaluation. Full size image The poor dendritic arborization and progressive death of PCs could be a consequence of the reduced number of cerebellar neurons that synapse onto the PC rather than an intrinsic defect in arborization. To investigate whether Snf2h is necessary for dendritic arborization and PC survival we further characterized the Snf2h cKO-PCP2 model, in which Snf2h loss is specific to PCs beginning at ~P10 (ref. 17 ). In this model, there is normal GNP proliferation resulting in a normally sized cerebellum and proper activation of post-mitotic markers in GCs and PCs, including Pax6 , Patched-1 and Gli-1 ( Supplementary Fig. 7a,c ). However, we observed a significant reduction of the PC apical dendritic arbor by P30 ( Fig. 7g,h ). Moreover, Snf2h cKO-PCP2 mice also display an ISWI dose-dependent increase in the total number of pyknotic PCs between P50 and P300 ( Supplementary Fig. 7b ). Similar results from both Snf2h cKO mouse strains allow us to conclude that Snf2h plays a cell-autonomous role in post-mitotic PC maturation and survival. Snf2h governs chromatin organization and histone H1 dynamics We reasoned that the progressive PC loss might result from altered chromatin architecture that impacts gene expression and compromises cell function. Indeed, studies in yeast and Drosophila have demonstrated multiple roles for ISWI complexes in chromatin compaction by repositioning nucleosomes to mediate linker DNA length and by facilitating histone H1 deposition [12] , [30] , [31] . To assess chromatin organization, we examined nuclear ultrastructure of cerebellar neurons by transmission electron microscopy (TEM). TEM images of E18.5 Snf2h cKO-Nes mice revealed that GNPs and PCs display numerous densely stained clumps within the euchromatin, a dispersed nucleolar region, chromatin loops and structures indicative of nuclear invaginations or micronuclei that collectively indicate that the chromatin structure is highly disorganized ( Fig. 8a ). Moreover, we observed that the altered chromatin organization is augmented in cDKO-Nes mice at E18.5 ( Fig. 8a , rightmost panel) and is progressive, both temporally and in a Snf2l-dose-dependent manner ( Fig. 8b–e ). Indeed, many pyknotic nuclei and cell ‘ghosts’ were clearly visible in Snf2h cKO-Nes mice by P21 ( Fig. 8c ). Collectively, these experiments demonstrate a progressive disorganization of the chromatin structure that correlates with the progressive death of GNPs and PCs, and the ataxic phenotype. 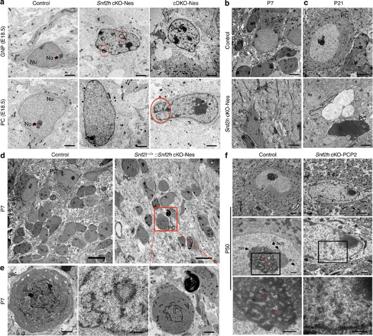Figure 8: Snf2h is necessary for proper chromatin folding. (a) Transmission electron microscopy (TEM) of GNPs and PCs through the cerebellar vermis fromSnf2hcKO-Nes, cDKO-Nes mice and control mice at E18.5. Red circles denote nuclear invaginations. GNP, granule neuron progenitor; PC, Purkinje cell; Nu, nucleus; No, nucleolus. Scale bars, 2 μm. (b,c) TEM fromSnf2hcKO-Nes and control mice through the cerebellum at P7 and P21. Note the abnormal morphology of mutant PCs and ‘cell ghosts’ in mutant cerebella. PC, Purkinje cell. Scale bars, 2 μm. (d,e) TEM through the cerebellar vermis from control andSnf2l−/+::Snf2hcKO-Nes mice at P7, revealing the aggravation of chromatin ultrastructure abnormalities within PCs upon additional removal of oneSnf2lcopy. Boxed area is enlarged in bottom rightmost panel. Scale bars, 10 μm (top panels); 2 μm (bottom panels). (f) TEM from P50Snf2hcKO-PCP2 mice and control littermates through the cerebellar vermis. Higher magnification images are provided in descending panels. Note the loss of nucleolar, heterochromatin and euchromatin ultrastructure and increased electron density, evidenced as ‘chromatin clumps’ within mutant PC nuclei. Stars denote nucleolar dense fibrillar centers (dfc). gc, granular centre; fc, fibrillar centre; no, nucleolus; eu, euchromatin; hch, heterochromatin. Scale bars, 2 μm (top panels); 500 nm (middle and bottom panels). At least three mice from each genotype were used for evaluation. Figure 8: Snf2h is necessary for proper chromatin folding. ( a ) Transmission electron microscopy (TEM) of GNPs and PCs through the cerebellar vermis from Snf2h cKO-Nes, cDKO-Nes mice and control mice at E18.5. Red circles denote nuclear invaginations. GNP, granule neuron progenitor; PC, Purkinje cell; Nu, nucleus; No, nucleolus. Scale bars, 2 μm. ( b , c ) TEM from Snf2h cKO-Nes and control mice through the cerebellum at P7 and P21. Note the abnormal morphology of mutant PCs and ‘cell ghosts’ in mutant cerebella. PC, Purkinje cell. Scale bars, 2 μm. ( d,e ) TEM through the cerebellar vermis from control and Snf2l−/+::Snf2h cKO-Nes mice at P7, revealing the aggravation of chromatin ultrastructure abnormalities within PCs upon additional removal of one Snf2l copy. Boxed area is enlarged in bottom rightmost panel. Scale bars, 10 μm (top panels); 2 μm (bottom panels). ( f ) TEM from P50 Snf2h cKO-PCP2 mice and control littermates through the cerebellar vermis. Higher magnification images are provided in descending panels. Note the loss of nucleolar, heterochromatin and euchromatin ultrastructure and increased electron density, evidenced as ‘chromatin clumps’ within mutant PC nuclei. Stars denote nucleolar dense fibrillar centers (dfc). gc, granular centre; fc, fibrillar centre; no, nucleolus; eu, euchromatin; hch, heterochromatin. Scale bars, 2 μm (top panels); 500 nm (middle and bottom panels). At least three mice from each genotype were used for evaluation. Full size image To confirm the cell-autonomous nature of the chromatin disorganization, we once again made use of Snf2h cKO-PCP2 mice. Sections from P50 mice were examined for chromatin ultrastructure changes by TEM. Similar to Snf2h cKO-Nes mice, we observed chromatin disorganization and loss of nuclear and nucleolar ultrastructure in P50 sections processed for TEM from Snf2h cKO-PCP2 but not from WT littermates ( Fig. 8f ). The temporal increase in densely stained clumps and disorganized nucleolar structures likely contribute to the dramatic increase in deregulated gene expression we observed between P0 and P10. To address this we investigated whether any global perturbations in histone modifications occur during this time. Indeed, P9 immunoblots of acid-extracted histones from Snf2h cKO-Nes and control mice identified a significant decrease in histone marks for active transcription including H3K4Me3 and H3K18Ac, and for transcriptional elongation (H3K36Me2), but not for the repressive mark H3K9Me3 ( Fig. 9a ). We additionally found that the histone variants H2A.Z and macro-H2A, which mark regions of active or repressed chromatin, respectively, were normal at P2 but were markedly reduced in mutant cerebella by P9 ( Fig. 9b ). These results suggested that altered gene expression likely arises from a defect in establishing specific chromatin domains. 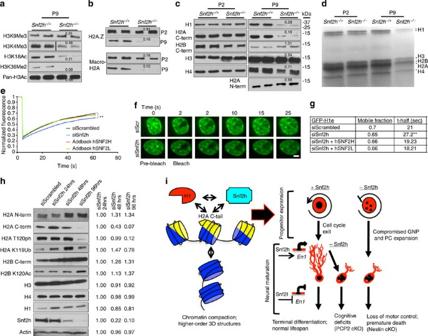Figure 9: Snf2h mediates chromatin transitions through linker histone H1 dynamics. (a,b) Immunoblots of acid-extracted cerebellar histones fromSnf2hcKO-Nes (Snf2h−/−) and control littermates (Snf2h−/+) for (a) histone H3 post-translational modifications at P9; or (b) histone variants H2A.Z and macro-H2A at P2 and P9. Values denote average densitometry relative to control samples (n=4). (c) Immunoblots of core histones from P2 and P9 cerebellar extracts fromSnf2hcKO-Nes and control littermates. Values denote average densitometry relative to control samples (n=4). (d) Colloidal blue staining of isolated P2 and P9 histones fromSnf2hcKO-Nes and control littermates to examine stoichiometry. (e) Mean normalized GFP-H1e FRAP curves of siScrambled (siScr); siSnf2h; siSnf2h+addback human (h) SNF2H; or siSnf2h+addback hSNF2L from transiently transfected mouse Neuro2A cells 48 h after treatment. A significant difference between recovery curves of siScrambled and siSnf2h is indicated. **P=0.008,n=20, Student’st-test. Error bars were omitted for clarity. (f) FRAP images of GFP-H1e from siScr (top) or siSnf2h (bottom) Neuro2A treated cells at the indicated times. Scale bar, 1 μm. (g) Mobile fractions and t-half values for GFP-H1e FRAP experiments. **P=0.008,n=20, Student’st-test. (h) Histone immunoblots of Neuro2A cells treated with siScr or siSnf2h for the indicated times. Snf2h KD is observed by 48 h. Actin served as loading control. Values denote average densitometry relative to siSnf2h 24 h treatment. (n=4). (i) Proposed model of Snf2h-dependent chromatin organization. Left, Snf2h interacts with the C-terminal tail of H2A to mediate histone H1 deposition and promote higher-order chromatin compaction and terminal differentiation32. Right-top, Snf2h is required for normal progression through the cell cycle35,37.Snf2hcKO-Nes mice have compromised expansion of the GNP and PC progenitor pools resulting in cerebellar atrophy. Right-bottom, after cell cycle exit, Snf2h- and Snf2l-dependent chromatin remodelling drives the establishment and maintenance of gene expression profiles. The co-regulation at theEn1locus is depicted as an example and this regulation promotes neural maturation. The embryonic removal of Snf2h (Nestin model) results in cerebellar hypoplasia and reduced dendritic arborization of PCs, causing severe ataxia and premature death. Similarly, Snf2h ablation in PCs (PCP2 model) also affects PC arborization, but conversely results in cognitive deficits rather than motor alterations. Figure 9: Snf2h mediates chromatin transitions through linker histone H1 dynamics. ( a,b ) Immunoblots of acid-extracted cerebellar histones from Snf2h cKO-Nes ( Snf2h −/− ) and control littermates ( Snf2h −/+ ) for ( a ) histone H3 post-translational modifications at P9; or ( b ) histone variants H2A.Z and macro-H2A at P2 and P9. Values denote average densitometry relative to control samples ( n =4). ( c ) Immunoblots of core histones from P2 and P9 cerebellar extracts from Snf2h cKO-Nes and control littermates. Values denote average densitometry relative to control samples ( n =4). ( d ) Colloidal blue staining of isolated P2 and P9 histones from Snf2h cKO-Nes and control littermates to examine stoichiometry. ( e ) Mean normalized GFP-H1e FRAP curves of siScrambled (siScr); siSnf2h; siSnf2h+addback human (h) SNF2H; or siSnf2h+addback hSNF2L from transiently transfected mouse Neuro2A cells 48 h after treatment. A significant difference between recovery curves of siScrambled and siSnf2h is indicated. ** P =0.008, n =20, Student’s t -test. Error bars were omitted for clarity. ( f ) FRAP images of GFP-H1e from siScr (top) or siSnf2h (bottom) Neuro2A treated cells at the indicated times. Scale bar, 1 μm. ( g ) Mobile fractions and t-half values for GFP-H1e FRAP experiments. ** P =0.008, n =20, Student’s t -test. ( h ) Histone immunoblots of Neuro2A cells treated with siScr or siSnf2h for the indicated times. Snf2h KD is observed by 48 h. Actin served as loading control. Values denote average densitometry relative to siSnf2h 24 h treatment. ( n =4). ( i ) Proposed model of Snf2h-dependent chromatin organization. Left, Snf2h interacts with the C-terminal tail of H2A to mediate histone H1 deposition and promote higher-order chromatin compaction and terminal differentiation [32] . Right-top, Snf2h is required for normal progression through the cell cycle [35] , [37] . Snf2h cKO-Nes mice have compromised expansion of the GNP and PC progenitor pools resulting in cerebellar atrophy. Right-bottom, after cell cycle exit, Snf2h- and Snf2l-dependent chromatin remodelling drives the establishment and maintenance of gene expression profiles. The co-regulation at the En1 locus is depicted as an example and this regulation promotes neural maturation. The embryonic removal of Snf2h (Nestin model) results in cerebellar hypoplasia and reduced dendritic arborization of PCs, causing severe ataxia and premature death. Similarly, Snf2h ablation in PCs (PCP2 model) also affects PC arborization, but conversely results in cognitive deficits rather than motor alterations. Full size image Studies in Drosophila have shown that ISWI ablation leads to global chromatin decompaction and a reduction in histone H1 (refs 12 , 31 ). As such, we analysed core histone proteins by immunoblot from Snf2h cKO-Nes mice and control cerebella at P2 and P9. At P2, all core histones were present at levels equivalent to wild-type mice ( Fig. 9c ). In contrast, we observed a severe reduction in histone H1 but not the other core histones by P9 ( Fig. 9c,d ). Interestingly, we noted that the H2A C-terminal antibody showed reduced detection of H2A at P9 but the N-terminal antibody showed normal levels, as did its dimer partner H2B ( Fig. 9c,d ). While this suggests that the epitope recognized by the C-terminal H2A antibody might be masked, modified or proteolytically cleaved, it remains unclear why we are observing this differential effect. Recent studies have demonstrated that the C-terminal tail of histone H2A is required for histone H1 loading onto DNA and is also necessary for Snf2h-dependent nucleosome translocation [32] . Moreover, the reduced levels of H1 and the possibility that the H2A tail is modified or clipped in Snf2h cKO-Nes mice suggested that Snf2h regulates histone H1 dynamics. To decipher an in vivo role for Snf2h in H1 chromatin dynamics, we performed fluorescence recovery after photobleaching (FRAP) experiments using GFP-H1e-tagged constructs transfected into Neuro2A cells before Snf2h knockdown (KD) [33] , [34] . To avoid any non-specific effects of cell death upon acute Snf2h ablation, FRAP experiments were performed at the 48-h time point. The cell nucleus in both siScrambled (siScr) control and siSnf2h-treated cells appeared normal in size and shape at the time of the experiments ( Fig. 9f ). siSnf2h-treated cells displayed an increased ‘bleached depth’ that suggests that the pool of unbound H1 is increased in the mutant samples. In addition to an increase in the unbound fraction, there was also a subtle change in H1 dynamics as we observed an ~10% reduction in histone H1e-GFP mobility and an ~20% increase in the half-maximal recovery time (t-half) compared with siScr controls ( Fig. 9e–g and Supplementary Movies 7 and 8 ). To demonstrate that the observed effect was specific to Snf2h, we restored the mobility of GFP-H1e by co-transfecting hSNF2H (addback hSNF2H) that is unaffected by the siRNA treatment ( Fig. 9e,g and Supplementary Movie 9 ). Conversely, Snf2l KD did not alter GFP-H1e dynamics ( Supplementary Fig. 8c ). However, exogenous expression of hSNF2L was also able to rescue GFP-H1e dynamics following Snf2h KD (addback hSNF2L), which is indicative of the functional compensation we have observed in Snf2h cKO-Nes mice ( Fig. 9e,g and Supplementary Movie 10 ). These studies suggest that Snf2h participates in the loading of histone H1 onto chromatin. We next investigated whether acute KD of Snf2h by siRNA treatment in Neuro2A cells could recapitulate the chromatin changes we observed in the Snf2h cKO mice. We observed a significant KD of Snf2h by 48 h and >90% loss by 96 h ( Fig. 9h ). We next analysed the cells for changes in nuclear morphology after DAPI staining. We observed a subtle reduction in the number of DAPI dense foci at 48 h and this preceded activation of phosphorylated Caspase-3, which was only detectable at 96 h after siSnf2h KD ( Supplementary Fig. 8a,b ). Despite significant Snf2h KD we only observed a modest ~20% decrease in histone H1 by 96 h after siSnf2h treatment ( Fig. 9h ). The core histones H3 and H4 showed no change, although we observed an unexplained increase in H2A and H2B protein levels. Similar to our results with the P9 cerebellar extracts, we observed a dramatic loss of H2A signal using the C-terminal H2A antibody ( Fig. 9h ). In addition, we also observed reduced signal with two H2A C-terminal tail modifications, namely phosphorylation of T120 and ubiquitination at K119 ( Fig. 9h ). While suggestive of a H2A C-terminal tail modification upon Snf2h loss, we were unable to identify the nature of such a change. Nonetheless, our studies indicate that an integral relationship between Snf2h, H1 and H2A is critical for chromatin folding and gene expression during cerebellar development ( Fig. 9i ). Ablation of Snf2h results in the loss of functional ACF/CHRAC, WICH and NoRC remodelling complexes that collectively have a major impact on the dynamics and organization of chromatin. Indeed, altered chromatin dynamics impaired cerebellar progenitor expansion, the transcription of key cerebellar patterning genes and the morphological maturation of PCs. As a result, Snf2h cKO-Nes mice developed cerebellar ataxia that resulted in their premature death, while Snf2h cKO-PCP2 had a normal lifespan, but displayed cognitive deficits and progressive PC death. A key feature of the developing post-natal cerebellum is the massive expansion of GNPs, a critical event in cerebellar foliation [24] . We demonstrate that the reduced cerebellar size in Snf2h cKO-Nes mice results from a combination of poor GNP and PC proliferation, without altering Shh signalling. Several studies have implicated ACF/CHRAC and WICH complexes in the replication of heterochromatin [19] , [20] . The WICH complex acts behind the replication fork to re-establish the local chromatin environment while the ACF/CHRAC complex is recruited as part of the DNA damage checkpoint response to collapsed replication forks [35] . Indeed, defective replication of heterochromatin is known to result in DNA damage, mitotic catastrophe and cell death, which can have a significant effect on cell number during the proliferative phase of tissue growth [36] , [37] . This would be consistent with our findings of increased TUNEL staining in Snf2h cKO-Nes mice at the onset of GNP expansion. Similarly, RNAi depletion in HeLa or U2OS cells results in increased apoptosis 24 h after SNF2H or ACF1 protein expression was strongly reduced [37] , [38] . Nonetheless, several alternative explanations exist that could account for the decreased growth of the cerebellum. Reduction of histone H1 may be sufficient to induce cell cycle arrest, as found with H3 ablation studies in yeast [39] . Similarly, reduced expression of Engrailed and/or other GNP or PC-specific TFs may impair growth, particularly since mouse models null for Pax6 , Math1 , NeuroD1 , En2 or En1 result in cerebellar hypoplasia [40] , [41] , [42] , [43] . Regardless, our experiments demonstrate a requirement for Snf2h in the proliferation of GNPs and PCs and the subsequent foliation of the cerebellum during the post-natal period. Purkinje neurons are critical for cerebellar function and we demonstrate that Snf2h is important for the maturation and function of this cell type. We show that dendritic arborization was compromised using two different Cre-driver lines (Nestin-Cre and PCP2-Cre) to ablate Snf2h. In the Snf2h cKO-Nes model, the poor arborization resulted in severe motor deficits that we attribute to the combined loss of both PCs and GCs. Conversely, the Snf2h cKO-PCP2 model presented with cognitive abnormalities reminiscent of the Purkinje-specific Tsc1 mouse strain with autistic-like features [44] . Indeed, dendritic defects and aberrant synaptic plasticity are common phenotypes for mouse strains inactivated for chromatin remodelling proteins [45] , [46] . Recent evidence shows that epigenetic regulation of synaptic plasticity extends beyond development, since electrophysiological deficits can be rescued by re-introduction of the missing CRC subunit in post-mitotic neurons [47] . Similar studies are required to dissect the individual roles of Snf2h -associated subunits to PC synaptic physiology and cognitive functions. In this regard, we are currently exploring whether environmental enrichment or in vivo re-introduction of Snf2h can rescue the motor dysfunction in Snf2h cKO-Nes mice. We surmise that the dendritic defects arise from aberrant transcription of target genes, particularly given the rampant increase in deregulated genes between birth and P10 (110 genes at P0 versus ~2,900 genes at P10). High-throughput ChIP-Sequencing studies from Drosophila and mouse cell lines indicate that ISWI and Snf2h interact at genes ~300 bp downstream of the transcriptional start site where it localizes nucleosomes into positions that stabilize a transcriptional (active or repressed) state [25] , [48] . Indeed, we observed enrichment for both Snf2h and Snf2l in a similar position at the En1 locus. The specific positioning of nucleosomes by Snf2h may also facilitate the loading of H2A.Z in progenitors, which acts to ‘poise’ genes for expression upon differentiation [4] . An inability to position nucleosomes around the promoter or exchange H2A for H2A.Z or macro-H2A may account for the poor regulation we observed for many genes by P10. It is also possible that Snf2h and Snf2l impart exquisite transcriptional control on developmentally important genes, as suggested by the function of known targets [13] , [49] , [50] . For example, Foxg1 levels determine whether a progenitor undergoes self-renewal or differentiation [51] and Snf2l mutant mice had increased Foxg1 expression that enhanced progenitor proliferation and increased brain size [13] . Similarly, the interaction of both Snf2h and Snf2l at the En1 gene (co-modulation) may regulate its expression levels and/or recruitment to target loci to control PC maturation, as has been observed for the TF Olig2 and the chromatin remodeller Brg1 during oligodendrocyte differentiation [52] . We propose that Snf2h poises and/or triggers the En1 locus for activation, while Snf2l is turned on during late cerebellar development to tightly modulate (i.e. repress) En1 levels in the mature PC. Certainly, the interaction at co-modulated target genes may facilitate rapid and dynamic changes in gene expression induced by extrinsic signals. Genome wide epigenetic profiling experiments have supported the hypothesis that neurogenesis is accompanied by the transition of a highly dynamic chromatin environment within progenitor cells to a more restrictive epigenetic landscape that dictates gene expression programmes specific to each lineage [2] , [3] . Chromatin condensation is dependent on nucleosome repeat length and the incorporation of the linker histone H1 (ref. 6 , 7 ). In vitro studies have shown that ISWI protein complexes assemble and evenly space nucleosomes on a chromatin template [11] , while loss of ISWI function in Drosophila results in reduced histone H1 levels and the decondensation of the X chromosome [12] , [30] , [31] . Other studies have noted a requirement for NoRC in the formation of perinucleolar heterochromatin structures [53] . In this regard, we observed a wide range of chromatin changes in Snf2h cKO mice both by TEM and immunoblot including patches of condensed euchromatin, loss of histone H1, altered levels of specific histone marks and histone variants, and disorganized nucleolar structures that collectively indicate that chromatin organization is abnormal. As discussed above, aberrant heterochromatin formation during replication could lead to mitotic catastrophe and cell death of the GNPs, thereby accounting for the cerebellar hypoplasia we observed. In addition, aberrant nucleosome spacing and maintenance of nucleosome-free regions could disrupt gene expression programs that could result in the maturation defects we observed and the progressive cell death, perhaps initiated in a cell with an inability to respond to an external signal. While we favour the idea that Snf2h loss promotes changes in chromatin structure directly, resulting in an inability to function and subsequent death, we cannot rule out that the chromatin disorganization we observed in Snf2h-null cells is indirect and representative of cells that were in the early stages of programmed cell death. Future studies will aim to distinguish between these possibilities. Higher-order chromatin packaging is dependent on histone H1 as embryos lacking three histone H1 subtypes (H1c, H1d and H1e) die by mid-gestation with a broad range of defects [54] . Histone H1 has been shown to play a key role in silencing gene expression by tethering Su(var)3–9 to heterochromatin [55] . Unlike core histones, which display very slow kinetics with residence time in the range of hours, linker histones are highly mobile, and more recently were shown to have metastable states with partially bound molecules [56] , [57] . Indeed, H1 dynamics reflects cell plasticity and chromatin compaction in general [33] . This may explain the modest ~10% reduction in H1e-GFP mobility observed upon Snf2h depletion in Neuro2A cells. Whereas this mobility was restored upon hSNF2H or hSNF2L overexpression, these measurements may only reflect the unbound H1 pool. Nonetheless, our evidence suggests that Snf2h loss results in abnormal higher-order chromatin packaging that disrupts genome organization and chromatin fluidity. Recent studies have demonstrated that the C-terminal tail of histone H2A is required for histone H1 loading and for Snf2h-dependent nucleosome translocation [32] . Indeed, the altered H1 levels and abnormal H2A post-translational processing in Snf2h cKO-Nes mice is suggestive of a functional relationship between Snf2h, histone H1 and H2A. We propose that an interaction between H2A and Snf2h may alter the accessibility of the H2A C-tail for loading histone H1 onto chromatin to facilitate chromatin packaging. In this regard, biochemical studies have shown that removal of the H2A C-tail increased the mobility of nucleosomes in vitro [32] , [58] . Such a mechanism for increasing the mobility of the nucleosome may be a compensatory response in the Snf2h cKO mice to facilitate nucleosome spacing and chromatin compaction, a function normally provided by Snf2h-dependent chromatin remodelling. In addition, Snf2h interactions with the H2A tail could promote H2A/H2B dimer removal and subsequent H2A variant exchange to activate and/or repress gene activity. Within progenitor cells these functions could mark genes for expression (H2A.Z loading) or repression (macro-H2A loading) upon differentiation, while establishing the restrictive chromatin landscape (through histone H1 loading) that accompanies the transition from progenitor expansion to terminal differentiation [59] , [60] . While exciting, such mechanisms remain speculative and the exact relationship between Snf2h loss and H2A C-tail post-translational processing remains to be deciphered with more biochemical studies. Indeed, delineating the epigenetic regulation of neuronal development is crucial to our understanding of intellectual-disability disorders caused by mutations in epigenetic modifying enzymes. As a whole, our findings highlight the complexity and functional diversity of Snf2h-containing CRCs during brain development, and their roles in controlling chromatin organization as cells modulate their chromatin environment from a ‘largely open’ progenitor state to the ‘highly restricted’ state of a fully differentiated neuron during cerebellar morphogenesis and neural maturation ( Fig. 9i ) [60] . Generation of Snf2h fl/fl mice Snf2h exon5fl/exon5fl ( Snf2h fl/fl ) mice were generated through homologous recombination in WW6 ES cells as described [14] . Briefly, a 6.0-kb fragment of the Snf2h gene containing exons 4–8, into which loxP sites were inserted 5′ and 3′ of exon 5, was cloned into the pEasyFlirt vector (a gift of Dr M.P. Lisanti, University of Manchester, UK). This vector has a neomycin resistance gene flanked by Frt sites, which was removed in mice generated from correctly targeted ES cells by breeding to Flp1 recombinase mice [61] . Snf2h fl/fl mice were viable, fertile and did not exhibit any gross behavioural abnormalities. Cre-mediated deletion of Snf2h exon 5 was tested by breeding to ZP3-Cre mice [62] for which embryos homozygous for a deleted exon 5 died in utero due to abnormal progenitor expansion, as previously described [14] . Mouse breeding Snf2h fl/fl mice were backcrossed for six generations to a C57Cl/6 background and bred with a C57Bl/6 Nestin-Cre −/+ driver line [16] that also carried a Snf2h null allele [14] , thereby generating Snf2h cKO-Nes mice ( Snf2h − /fl ::Nes-Cre −/+ ). We also bred Snf2h fl/fl mice to the PCP2-Cre driver line [17] that lived normally into adulthood and showed no gross behavioural abnormalities. For Snf2l ablation, we used the previously characterized Ex6Del line [13] for breeding, thus generating Snf2l-/y::Snf2h cKO (cDKO-Nes) and Snf2l−/y::Snf2h cKO-PCP2 (cDKO-PCP2), as well as Snf2l−/+::Snf2h cKO-Nes and Snf2l−+::Snf2h cKO-PCP2 compound heterozygotes. For embryo staging, embryonic day 0.5 (E0.5) was defined as noon on the day of vaginal plug detection. Animals were kept in an animal house under specific pathogen-free conditions in a 12/12 light:dark cycle with water and food ad libitum. The University of Ottawa Animal Care and Use Committee approved all experiments. C57Bl/6 and FVBN/J wild type mice were purchased from Charles River (Montreal, QC, Canada). PCP2-Cre mice were obtained from The Jackson Laboratory (Stock no. 004146; Bar Harbor, ME, USA). Behavioural analysis All behavioural tests were completed in the Behavior Core Facility at the University of Ottawa using standardized protocols. Animals were habituated to the testing room at least ~1 h before testing. Behavioural assays were performed irrespective of sex for Snf2h cKO-Nes mice and tested between P20-P25. For Snf2h cKO-PCP2 mice, female and male mice were assessed independently at 4–6 months of age, for which we did not observe sex-specific differences in behaviour and pooled the data. For behavioural assays, one-way ANOVA was used for at least 10 mice per genotype. The values are presented as the mean±s.e.m. Suspended wire test Mice were suspended by their forepaws on a 2 mm wire, and the amount of time they remained on the wire was recorded. Dowel test Mice were placed in the centre of a horizontal pole (1 cm diameter) and the time mice remained on the pole was recorded. If mice walked across and off the dowel, they were placed back onto the dowel. Trials lasted for a maximum of 2 min. Elevated platform Mice were placed in the centre of a 15-cm 2 round elevated platform 50 cm above the ground and the time mice remained on the platform was recorded. Student’s t -test was used for statistical significance. Rotarod Mice were trained and tested on the accelerated rotarod (rod diameter 3 cm) for 300 s for five times before measurements (IITC, Woodland Hills, CA, USA). Starting speed was set at 4 r.p.m. and maximum speed at 40 r.p.m. The latency to fall from the rotarod was recorded. If animals were able to stay on the rod for 300 s, the latency to fall recorded was 300 s. The animals received four trials per day, with a trial interval of 30 min, for 2 consecutive days. Pole test Mice were placed head-upward on the top of a rough surfaced vertical pole (8 mm diameter × 55 cm tall) and the time for descending recorded. The time required for the mouse to turn downward after placing and the total time on the pole until the mouse reaches the bottom is recorded. Mice were trained for 2 days before test. Five trials were averaged on day 3. Open field Animals were placed in the centre of a 45 × 45 × 45-cm chamber equipped with photobeams (Accuscan) to record activity during a 10-min test period. Elevated plus maze Animals were habituated to the test room for at least 2 days before test. Animals were placed in the centre of a maze consisting of two arms (each arm 5 cm wide × 60 cm long) enclosed by ~15-cm-high walls, and two open arms (each arm 25 × 7.5 cm, with a raised 0.5 cm lip at edges) elevated 1 metre above ground and with equidistant arms from the centre of the platform. The amount of time the animals spent in the open or closed arms, the total number of entries and the total distance travelled were recorded for 10 min using video detection software (Ethovision, Wageningen, Netherlands). Social interactions A control mouse is placed in the corner of an open field box (under dim red light) that measures 45 cm long on each side × 45 cm high and containing a 5.5 × 9.6 cm wire mesh rectangular cage. The mouse is given 5 min to explore the arena and then removed. A few seconds later, a test mouse (or social target) of the same strain, age and gender is placed inside the rectangular wire mesh cage and the control mouse placed back in the arena. The time the social target interacts with the control mouse in 5 min trials is recorded using Ethovision 7 XT automatic tracking software. Total distance travelled, time spent in two corners across the wire mesh cage and velocity is also recorded. Fear conditioning On the first day (training), the animal is placed in the fear-conditioning apparatus for a total of 6 min. After the first 2 min in the apparatus a tone is played for 30 s ending with a 2-s shock. One minute following the shock, the tone is played again for 30 s ending with a 2-s foot shock. For the remaining 2 min there is no tone or shock. The freezing behaviour of the animal is recorded throughout the 6 min. This is the training in which the mouse receives two exposures to the tone followed by the shock and this occurs in a novel context, which is the conditioning box. On the second day, contextual conditioned fear testing begins. This measures the fear associated with being in the same environment where the shock was delivered (done ~24 h after training). The mouse is placed in the same apparatus with all the same lighting and room conditionings for 6 min and freezing behaviour is recorded. BrdU-birthdating Timed-pregnant females were injected intraperitoneally with 100 μg per g body weight of 5-bromo-2′-deoxyuridine (BrdU; Sigma) and pups killed at indicated times. For BrdU-pulse labelling, timed-pregnant females were injected with BrdU and killed 90 min later. For BrdU immunodetection, sections were incubated in 2 N HCl for 10 min at 37 °C, rinsed in 0.1 M sodium borate (pH 8.3), blocked and incubated overnight at 4 °C with rat monoclonal anti-BrdU antibody 1:300 (Abcam no. 6326). The average number of immunopositive cells was determined from five separate fields under × 40 magnification in confocal Z-stacks (or cubic bins) of 18 × 10 3 μm 3 . TUNEL assay Sections were examined for DNA fragmentation with the TUNEL in situ cell death detection kit (Roche Applied Science, ON, Canada) according to the manufacturer’s instructions. The average number of TUNEL-positive cells was determined from five separate fields under × 40 magnification in cubic bins. Golgi–Cox staining Golgi staining was completed using FD Rapid GolgiStain Kit (FD NeuroTechnologies). Briefly, P20 mice were intracardially perfused with 4% paraformaldehyde (PFA) in 0.1 M PBS and stained according to the manufacturer’s instructions. Tissues were sectioned at 60–100 μm and mounted on gelatin-coated slides. Immunofluorescent histochemistry For embryonic tissue, 16–20 μm sections were used. For post-natal brains, 40–50 μm free-floating sections were used. Sections were washed four times in PBST (PBS with 0.1% Triton X-100), blocked (1 h, room temperature (RT)) in 10% horse serum/PBST, and incubated (overnight, 4 °C) in primary antibodies. The following primary antibodies were used from Abcam: rabbit anti-Snf2h (1:500, no. 72499); rabbit anti-Snf2l (1:100, no. 37003); mouse anti-NeuroD1 (1:500, no. 60704); rat anti-BrdU (1:300; no. 6326) and rabbit anti-Engrailed (1:500; no. 32817). Mouse anti-calbindin (1:200, Sigma C9848); rabbit anti-calbindin (1:300, Sigma C2724); rabbit anti-GFP (1:1,000, Molecular Probes); mouse anti-BrdU (1:100, DAKO); rabbit anti-phospho histone H3 (pH3; 1:200; Millipore no. 06-570); rabbit anti-Pax6 (1:200; Covance no. PRB-278P); mouse anti-NeuN (1:200, Millipore no. MAB377) and rabbit anti-pan-Engrailed (gift of Dr Alexandra Joyner, Memorial Sloan-Kettering Cancer Center, NY, USA). The following day, sections were washed five times in PBST and incubated (2 h, RT) with DyLight 488 , DyLight 594 or DyLight 649 -conjugated mouse pre-adsorbed secondary antibodies (1:1,000, Jackson Immunoresearch, PA, USA) against the IgG domains of the primary antibodies. All sections were counterstained with the nuclear marker DAPI (Invitrogen). Sections were mounted on slides with Dako Fluorescence Mounting Medium (Dako Canada, ON, Canada). X-Gal staining Staged embryos were quickly dissected and rinsed in 0.1 M PBS (pH 7.4) and fixed in 4% PFA for 30 min. Embryos were then rinsed three times with 0.1 M PBS supplemented with 0.01% Triton X-100 and incubated for ~1 h in the dark with staining solution (2 mM MgCl 2 , 0.02% NP-40, 5 mM potassium ferricyanide, 5 mM potassium ferrocyanide and 0.01% sodium deoxycholate in 0.1 M PBS, pH 7.4). Staining solution was rinsed off three times with 0.1 M PBS and embryos post-fixed for 30 min in 4% PFA. In situ hybridization In situ hybridization was performed from E18.5 or P0 14–16 μm sections through the cerebellar vermis using digoxigenin (DIG)-labelled antisense RNA riboprobes prepared by in vitro transcription from linearized plasmids containing complete or partial cDNA sequences of the following mouse genes: Shh , Gli1 , Mycn , Ptch1 , Ccnd1 and Pax6 . Labelling of RNA probes with DIG-UTP was performed according to the manufacturer’s recommendations. Briefly, 1 μg of linearized template was transcribed in a total volume of 20 μl using T7 or T3 polymerase (Roche) and DIG-UTP (Roche) for 1 hour at 37 °C. The reaction products were precipitated, resuspended in 100 μl of 10 mM EDTA and stored at −20 °C. DIG-labelled RNA probes were diluted in hybridization buffer (50% formamide, 10% dextran sulphate, 1 mg ml −1 yeast RNA, 1 × Denhardt’s and 1 × salt) and denatured for 10 min at 70 °C. Sections were hybridized overnight at 65 °C in a humidified box. The slides were washed twice in 50% formamide, 1 × SSC, 0.1% Tween 20 at 65 °C for 30 min followed by two washes in MABT (100 mM maleic acid, 150 mM NaCl, pH 7.5, 0.1% Tween-20) for 30 min at RT. Sections were blocked for 1 h at RT in MABT containing 20% sheep serum (Sigma) and 2% blocking reagent (Roche). The blocking solution was then replaced with blocking solution containing a 1:1,500 dilution of alkaline-phosphatase-conjugated Fab fragments of sheep anti-DIG antibodies (Roche) and the slides were incubated overnight at 4 °C in a humidified box. Slides were washed five times in MABT for 20 min at RT, twice in staining buffer (100 mM NaCl, 50 mM MgCl 2 , 100 mM Tris pH 9.5 and 0.1% Tween-20) and incubated for 1–5 h in staining buffer containing 10% polyvinyl alcohol, 4.5 μl ml −1 NBT and 3.5 μl ml −1 BCIP (Roche) in the dark at RT. Slides were washed several times in 1 × PBS and mounted in 50:50 glycerol:PBS. Western blotting Cerebellar or hindbrain (for E12 and E17 time points only) extracts were quickly dissected from individual pups and snap-frozen in dry ice. Cerebella were then homogenized in ice-cold RIPA buffer supplemented with protease inhibitor cocktail (Sigma) and incubated for 20 min on ice with gentle mixing. After pre-clearing by centrifugation (15 min at 17,000 g ), proteins were quantified by the Bradford method. Protein samples were resolved on sodium dodecyl sulphate polyacrylamide gels under denaturing conditions or using Bis-Tris 4–12% and Tris-Acetate 3–8% gradient gels (NuPage, Invitrogen) and blotted onto PVDF membranes (Immobilon-P; Millipore, MA, USA) by wet transfer for 1–2 h at 90 V. Membranes were blocked (45 min, RT) with 5% skim milk in TBST (Tris-buffered saline containing 0.05% Triton X-100), and incubated (4 °C, overnight) with the following antibodies: rabbit anti-Snf2h (1:4,000; Abcam no. 72499); sheep anti-Snf2l (1:2,000) [63] ; mouse monoclonal anti-Snf2l 1:1,000 (Alvarez-Saavedra and Picketts, unpublished); mouse anti-ß-actin (1:30,000, Sigma); rabbit anti-Engrailed-1 (1:2,000, Millipore) or mouse anti-Engrailed 4G11 (1:20, Developmental Studies Hybridoma Bank). Membranes were incubated (1 h, RT) with ImmunoPure HRP-conjugated goat anti-rabbit or goat anti-mouse IgG (H+L) secondary antibodies (1:50,000; Pierce, Rockford, IL, USA). Membranes were washed 5 × 5 min in TBST after antibody incubations, and the signal was detected using the Pierce Supersignal West Fempto chemiluminescence substrate (Pierce). Western blots were quantified using ImageJ software ( rsbweb.nih.gov/ij/ ). At least four individual lanes from multiple litters were used for quantification. All original western blots are shown in Supplementary Fig. 9 . Chromatin immunoprecipitation Cerebella was isolated from C57Bl/6 wild-type mice and cell pellets resuspended in 50 mM HEPES-KOH, pH 7.5, 140 mM NaCl, 1 mM EDTA, 1% Triton X-100, 0.1% sodium deoxycholate, 0.1% SDS and protease inhibitor cocktail and incubated on ice for ~30 min. Cells were then sonicated for 100 cycles (30 s pulse, 30 s rest intervals) to an average size of ~500–800 bp using a 4 °C sonicator (Bioruptor UCD-200, Diagenode, Inc., Sparta, NJ, USA). After sonication, cell debris was pelleted by centrifuging 2 min, 4 °C at 8,000 g . Supernatant was collected and a 20 μl input sample was analysed on a 2% agarose gel to verify chromatin size. Additionally, 100 μl of recovered chromatin was used for DNA quantification and as qPCR positive control (Input). GammaBind Plus Sepharose Beads (GE Healthcare, Piscataway, NJ, USA; Cat. No. 17-0886-01) were blocked with BSA (100 ng μl −1 beads; New England Biolabs, Ipswich, MA, USA) and salmon sperm DNA (100 ng μl −1 beads; Invitrogen) for 30 min at RT. Beads were washed three times with RIPA buffer (50 mM Tris–Cl, pH 8, 150 mM NaCl, 2 mM EDTA, pH 8, 1% NP-40, 0.5% sodium deoxycholate, 0.1% SDS with protease inhibitor cocktail) and resuspended in two volumes of RIPA. Pre-clearing of recovered chromatin was performed by incubating with 100 μl of blocked GammaBind Plus Sepharose Bead slurry for 30 min at 4 °C. Beads were centrifuged for 2 min, 4 °C at 8,000 g , and pre-cleared chromatin was recovered and further diluted 1:10 in RIPA for IP. IP was performed overnight at 4 °C by incubating ~50 μg of pre-cleared chromatin with 2 μg of the following rabbit antibodies from Abcam: anti-Snf2h; anti-Snf2l; anti-histone H3; or rabbit IgG (Jackson Immunoresearch). We also used anti-H3K9Ac; and anti-H3K9Me3 as internal controls. Immune complexes were captured with 120 μl of blocked GammaBind Plus Sepharose Bead slurry for 2 h at 4 °C. Beads were then collected by centrifuging for 2 min at 8,000 g . Beads were washed three times with 20 mM Tris–Cl, pH 8, 150 mM NaCl, 0.1% SDS, 1% Triton X-100 and 2 mM EDTA, pH 8, and once with 20 mM Tris–Cl, pH 8, 500 mM NaCl, 0.1% SDS, 1% Triton X-100 and 2 mM EDTA (pH 8). DNA was eluted with 150 μl of elution buffer (1% SDS, 100 mM NaHCO 3 ) for 15 min at RT. Eluted DNA was further diluted in two volumes of elution buffer and incubated overnight at 65 °C with 100 μg of proteinsase K (Invitrogen) for crosslink reversal. The DNA was phenol–chloroform-extracted and resuspended in 100 μl of TE, pH 8 (10 mM Tris–Cl, pH 8, 1 mM EDTA, pH 8). In all, 1 μl (1/100th) of DNA was used per reaction for quantitative PCR analysis. Triplicate or quadruplicate samples were ran per reaction and three independent ChIP experiments were carried out per time point. Primers are listed in Supplementary Table 1 . Quantitative real-time PCR For qPCR analysis of ChIP DNA, PCRs were carried out using the SYBR Green Advantage qPCR premix (Clontech) and run under the following conditions: one cycle at 95 °C for 1 min, 45 cycles at 95 °C for 10 s, 60 °C for 10 s and 72 °C for 20 s. All primers were analysed by melt curve analysis and agarose gel electrophoresis after qPCR amplification. Primers are listed in Supplementary Table 1 . The ΔΔCt method was used to compare fold-change. L32 was used as internal control. Triplicate or quadruplicate samples were ran per reaction and a minimum of three mice were analysed per genotype. Student’s t -test was used for statistical significance. Reverse transcription Cerebella were quickly dissected from mutant and control littermates and RNA was isolated using Trizol (Invitrogen) according to the manufacturer’s instructions. Glycogen (Ambion) was used as carrier. One microgram of total RNA was reverse-transcribed using random primers and SuperScriptIII (Invitrogen). cDNA was further diluted 1:20 and 1 μl was used per qPCR (described above). RNA integrity is shown in Supplementary Fig. 9 Microarrays Gene expression profiling was performed on RNA isolated from dissected cerebella tissue of P0 or P10 Snf2h cKO-Nes and wild-type control mice. RNA samples were labelled with Cy5 or Cy3 using 3DNA Array 900 kits (Genisphere, Hatfield, PA, USA) following the manufacturer’s instructions. Snf2h cKO-Nes and control samples were then cohybridized to MEEBO 38.5K arrays (Microarrays Inc., Huntsville, AL, Canada). A total of four replicates were performed for P0 and three for P10 and in both cases the labelling dyes were flipped for at least one replicate to counter dye bias. Probe-specific signals were quantified using the ScanArray express (Perkin Elmer, Waltham, MA). On the resulting raw background subtracted signals intra-array normalization (correcting for Cy5/Cy3 bias) was performed with global loess, inter-array normalization with the quantile method and statistical analysis via the WEBARRAY online tool ( http://www.webarraydb.org/webarray/index.html ). M (log 2 ratio of Snf2h cKO/control signal) and A values (log 2 average signal strength) were then determined for all probes. A probe (gene) was scored as differentially expressed on an array if it demonstrated a P -value <0.01, and had sufficient detectable signals across all replicates (A value (log 2 ) >7). Microarray filtering Cell-type-specific gene expression from P0 and P10 Snf2h cKO-Nes cerebellar arrays was determined by comparing the differentially expressed genes with the cell-type-specific gene expression lists from publicly available RNA-Seq data from adult cerebellar PCs, GCs and BG [26] . The unique gene identifiers of the differentially expressed genes from our arrays and from the RNA-Seq datasets were converted to MGI-approved gene symbols. This conversion ensures that genes presented with synonyms are not missed during the comparisons. The MGI symbols from the differentially expressed genes in our arrays were compared with each cell-type-specific gene list and reported as differentially expressed genes from Snf2h cKO-Nes cerebella in the corresponding cell types. Image acquisition and processing Tissue sections were examined and images captured using a Zeiss 510 laser scanning confocal microscope with UV (405 nm), argon (488 nm), helium/neon (546 nm) and helium/neon (633 nm) lasers. All images were acquired as 10–30 μm Z-stacks (in 1–2 μm intervals) and analysed as projections using the LSM 510 Image Browser software (Zeiss, Oberkochen, Germany). Epifluorescent and light microscopy images were acquired with a Zeiss Axiovert Observer Z1 epifluorescent/light microscope equipped with an AxioCam cooled-color camera (Zeiss). Images were exported to Adobe Photoshop CS5 (Adobe Systems Inc., San Jose, CA, USA) and further processed for contrast when necessary. Acid-based histone extraction Histones were acid-extracted from P2 and P9 Snf2h cKO and control cerebella or from Neuro2A cells after siRNA treatment. Briefly, cerebellar tissue was quickly dissected and separated from the inferior and superior colliculi and brain stem and snap-frozen on dry ice. Then, tissue was homogenized in TEB+ buffer (0.1 M PBS, 0.5% Triton X-100, 5 mM sodium butyrate, 0.02% NaN3 complemented with protease inhibitors cocktail (Sigma)), lysed on ice for 20 min and centrifuged for 10 min at 2,000 r.p.m. at 4 °C. Then, the supernatant was discarded and the pellet resuspended in 0.2 N HCl at a cell density of 4 × 10 7 cells per ml overnight with stirring at 4 °C. Samples were then centrifuged for 10 min at 2,000 r.p.m. at 4 °C and supernatant containing free histones collected and quantified for western blotting. The following antibodies were used from Active Motif: anti-histone H1 1:4,000 (no. 61201); anti-H2A acidic patch N-terminal 1:4,000 (no. 39111); anti-H2A C-terminal (no. 39591); anti-H2A T120ph 1:2,000 (no. 61195); anti-H2B 1:4,000 (no. 39125); anti-H2B K120Ac 1:4,000 (no. 39119); anti-macro-H2A1 1:1,000 (no. 39593). From Abcam: anti-H3 1:30,000 (no. 1791); anti-H4 1:5,000 (no. 10158); anti-H2AZ 1:5,000 (no. 4174); anti-H3K4Me3 1:10,000 (no. 8580); anti-H3K9Me3 1:5,000 (no. 8898) and anti-H3K18Ac 1:5,000 (no. 1191). From Millipore: anti-H3K36Me2 1:1,000 (no. 07-274); anti-pan-H3Ac 1:5000 (no. 382158) and anti-H2A K119Ub1 1:2000 (no. 8240; Cell Signaling). In all, 3–5 μg of total histones were loaded onto 15% SDS–PAGE linear gels and immunoblotted as described above. All original western blots are shown in Supplementary Fig. 9 . Colloidal Blue Staining Kit (Invitrogen) was used to assess histone stoichiometry in 18% SDS–PAGE linear gels as indicated by the manufacturer. Vector construction Human SNF2L cDNA comprising the entire open reading frame (+exon1/−exon13/+NLS) was amplified from a pcDNA3 expression plasmid [64] in a two-step process. The 5′ end of SNF2L cDNA was amplified with SNF2L-EcoRI-Fwd (5′-TAAGGAATTCATGGAGCA-3′) and SNF2L-XhoI-Rev-internal (5′-ACCTCTCGAGCTATGT-3′) primers, followed by purification of the PCR products, restriction digest by EcoRI and XhoI, and directional subcloning into the pBRIT-LoxP-NTAP and pBRIT-LoxP-CTAP retroviral plasmid vectors, which have been previously described [65] . The remaining 3′ sequence of SNF2L was then subcloned non-directionally following amplification with SNF2L-XhoI-Fwd-internal (5′-ATAGCTCGAGAGGTAG-3′) and SNF2L-XhoI-Rev (5′-ATGCTCGAGGGATTTCACCTTCTTG-3′) primers and a restriction digest with XhoI. Similarly, SNF2H cDNA comprising the entire open reading frame was cloned into the pCI-neo expression vector (Promega Corp. Madison, WI, USA) then amplified with the SNF2H-BamHI-Fwd (5′-AAAAGGATCCATGTCGTCCGCGGCCGAGCC-3′) and SNF2H-XhoI-Rev (5′-AAAACTCGAGTAGTTTCAGCTTCTTTTTTCTTCC-3′) primers and directionally subcloned into the pBRIT-LoxP-NTAP and pBRIT-LoxP-CTAP vectors, following restriction digest with BamHI and XhoI. All clones were verified by sequencing at McGill University and Génome Québec Innovation Centre (Montreal, QC, Canada). siRNA knockdown on Neuro2A cells Neuro2A cells were freshly obtained from ATCC (Manassas, VA, USA) and grown in DMEM medium containing 10% FBS, L -glutamine and no antibiotics. Briefly, cells were grown to a confluency of ~80% and transfected using Lipofectamine 2000 (Invitrogen) with 75 nM siSnf2h (Thermo Scientific, Ottawa, ON, Canada; siGENOME, mouse Smarca5 , D-041484-03); 75 nM siScrambled (siGENOME non-targeting siRNA no. 1, D-001210-01-05); or 75 nM siSnf2l (OriGene Technologies, Inc, Rockville, MD, USA; Smarca1 (mouse) no. SR421862B). Total proteins or acid-extracted histones were collected as described above and analysed by immunoblotting. Fluorescence recovery after photobleacing Neuro2A cells were grown in DMEM medium containing 10% FBS, L-glutamine and 1 × penicillin/streptomycin. H1e-GFP plasmid has been previously described [34] . FRAP experiments were conducted essentially as described [33] . Cells were grown in eight-well μ-slides (ibidi LLC, Martinsried, Germany) and transfected with H1e-GFP plasmid together with 75 nM of each of the siRNAs using Lipofectamine 2000 (Invitrogen). For hSNF2H and hSNF2L ‘addback’ studies, pBRIT-FLAG-hSNF2H or pBRIT-FLAG-hSNF2L was added to the transfection mix. Photobleaching studies were performed using a Revolution spinning disk (CSUX, Yokogawa, Japan) and an EMCCD high-speed imaging system (Andor Technology, Belfast, UK) equipped with a FRAPPA module (Andor Technology) and with solid-state lasers mounted on an Olympus IX81 fully automated microscope. During the entire imaging process, cells were maintained under controlled CO 2 , temperature and humidity using an environmental chamber (Life Imaging Services, Basel, Switzerland). Bleaching was performed with a × 60 oil objective (NA=1.4). Images were captured every 250 ms using an EMCCD iXon+ camera (Andor, UK). Typically 240 post-bleach images were collected. Data from more than 20 cells were collected per experiment. All FRAP experiments were performed at least three times and plots for one representative experiment are shown. Data processing was performed using the easyFRAP program [66] , based on the double normalization method [67] . Curve fitting was performed using MATLAB’s non-linear least-squares function. The method to calculate fully normalized recovery curves has been described previously [68] . This method was used to estimate the mobile protein fraction and t-half of protein. Two-tailed Student’s t -test was used to compare the significance of differences between FRAP curves [69] . Transmission electron microscopy Cerebella (E18.5, P7 and P21) were collected under a stereomicroscope, cut into sections of 1–2 mm thickness through the cerebellar vermis region and fixed for at least 4 h to overnight in Karnovsky’s fixative (4% PFA, 2% glutaraldehyde and 0.1 M cacodylate in phosphate-buffered saline, pH 7.4) at 4 °C. These specimens were subsequently washed twice in 0.1 M cacodylate buffer for 1 h and once overnight at RT. Sections were then post-fixed with 1% osmium tetroxide in 0.1 M cacodylate buffer for 1 h at 4 °C, and washed twice for 5 min in water. The specimens were dehydrated twice for 20 min for each step in a graded series of ethanol from water through 30–50–70–85–95% ethanol and twice for 30 min in 100% ethanol (molecular sieves were used to dehydrate ethanol), followed by twice for 15 min in 50% ethanol/50% acetone and twice for 15 min in 100% acetone. Sections were infiltrated in 30% spurr/acetone for 15 h (overnight) then in 50% spurr/acetone for 6 h and in fresh 100% spurr resin overnight. Spurr was changed twice a day for 3 days at RT. All infiltration steps were carried out on a rotator. Sections were then embedded in fresh liquid spurr epoxy resin and polymerized overnight at 70 °C. Ultrathin sections (80 nm) from the cerebellar vermis were collected onto 200-mesh copper grids and allowed to dry overnight before staining. Grids were stained with 2% aqueous uranyl acetate and with Reynold’s lead citrate. Sections were observed under a transmission electron microscope (Hitachi 7100). All ultrastructural analyses were based on at least three mice per genotype of the same age for each group examined. Toluidine blue staining Semithin sections of 0.5 μm were stained with 1% toluidine blue and 2% borate in distilled water. Histological samples were scanned with a MIRAX MIDI automated scanning light microscope (Zeiss) and images processed with Zeiss MIRAX Viewer software (Zeiss). Statistics Group statistical analysis was performed via two-tailed Student’s t -test or one-way ANOVA, where indicated. P <0.05 was accepted as statistically significant. At least three mice per genotype were used for evaluation. Values are presented as the mean±s.e.m. How to cite this article: Alvarez-Saavedra, M. et al . Snf2h-mediated chromatin organization and histone H1 dynamics govern cerebellar morphogenesis and neural maturation. Nat. Commun. 5:4181 doi: 10.1038/ncomms5181 (2014). Accession codes: All raw and processed microarray data have been deposited into Gene Expression Omnibus under the accession number GSE42371 .